Pellino3 targets RIP1 and regulates the pro-apoptotic effects of TNF-α Tumour necrosis factor-α (TNF) can activate NF-κB to induce pro-inflammatory genes but can also stimulate the caspase cascade to promote apoptosis. Here we show that deficiency of the ubiquitin E3 ligase, Pellino3, sensitizes cells to TNF-induced apoptosis without inhibiting the NF-κB pathway. Suppressed expression of Pellino3 leads to enhanced formation of the death-induced signalling complex, complex II, in response to TNF. We show that Pellino3 targets RIP1, in a TNF-dependent manner, to inhibit TNF-induced complex II formation and caspase 8-mediated cleavage of RIP1 in response to TNF/cycloheximide co-stimulation. Pellino3-deficient mice also show increased sensitivity to TNF-induced apoptosis and greatly increased lethality in response to TNF administration. These findings define Pellino3 as a novel regulator of TNF signalling and an important determining factor in dictating whether TNF induces cell survival or death. TNF is a pro-inflammatory cytokine that can also regulate cell proliferation, differentiation and death [1] . The binding of TNF to its receptor TNFR1 leads to association of TNFR1-associated death domain protein (TRADD) [2] with the receptor complex and this initiates signal transduction pathways culminating in activation of the transcription factor NF-κB and the MAP kinase pathways [3] . Although NF-κB serves to protect cells from cell death, the activation of TNFR1 can also trigger activation of the caspase cascade resulting in cell death by apoptosis [4] . The outcome of TNF stimulation depends on the sequential formation of different signalling complexes upon binding of TNF to its receptor [1] , [5] , [6] , [7] , [8] . The initial association of TNFR1 with TRADD facilitates the further recruitment of a number of signalling molecules including receptor interacting protein 1 (RIP1), TNF receptor-associated factor 2 (TRAF2) or TRAF5 and the cellular inhibitor of apoptosis proteins (cIAPs) cIAP1 and cIAP2 to form a signalling complex called complex I (refs 6 , 9 , 10 ). This results in the K63 ubiquitylation of RIP1 by TRAF-2 (refs 11 , 12 , 13 , 14 ) and the cIAPs [15] , [16] , [17] leading to downstream activation of NF-κB. The activation of NF-κB is dependent on phosphorylation and degradation of its inhibitory IκB proteins. The phosphorylation of the latter is catalysed by the IκB kinase (IKK) complex consisting of two catalytic subunits IKKα and IKKβ and the scaffolding subunit IKKγ (also termed NFκB-essential modulator (NEMO)) [18] , [19] , [20] . Polyubiquitinated RIP1 allows for interaction with the ubiquitin-binding domain of IKKγ [21] , thus having an important role in the activation of NF-κB by recruiting the IKK complex to TNF-R1 (refs 22 , 23 ). The recruited IKK complex may be activated by the upstream kinase TAK1 that is also recruited to polyubiquitinated RIP1 via the ubiquitin-binding domains of TAK1-associated proteins termed TABs [24] , [25] , [26] . Thus, the K63 polyubiquitination of RIP1 is associated with downstream activation of NF-κB and the induction of anti-apoptotic genes such as cellular FLICE Inhibitory protein (c-FLIP) and cIAPs that prevent cell death [27] , [28] , [29] . However, NF-κB also upregulates A20 and CYLD, which remove K63-specific polyubiquitin chains from RIP1 and abolish its ability to activate NF-κB [4] , [30] , [31] . In its unubiquitinated form RIP1 can dissociate from TNFR1, with or without TRADD, to interact with Fas-associated death domain (FADD) protein that in turn recruits procaspase 8 to form an intracellular signalling complex (complex II), also called death-inducing signalling complex (DISC) [8] , [16] , [30] , [32] , [33] . The formation of complex II triggers processing and activation of caspase 8 leading to initiation of the caspase cascade and ultimately cell death. Furthermore, caspase 8 can also cleave RIP1 to further promote TNF-induced apoptosis [34] . RIP1 also has a key role in Toll-like receptor (TLR) pathways and mediates IKK activation in response to signalling by the TLR3 and TLR4 adaptor protein TRIF [35] , [36] . Genetic ablation experiments have shown Peli1 to be the E3 ubiquitin ligase for RIP1 in the TLR3/TLR4 pathways [37] . Peli1 belongs to the mammalian Pellino family of E3 ubiquitin ligases that is made up of four family members (Pellino1, Pellino2 and two spliced variants of Pellino3 (Pellino3s and 3l) [38] , [39] . Each member of the family contains a N-terminal forkhead-associated (FHA) domain, a phosphothreonine-binding module that facilitates interaction with IL-1R-associated kinases (IRAKs) [40] , and a C-terminal RING-like domain that catalyses K63 polyubiquitination of IRAKs [41] , [42] , [43] . The latter are key signalling intermediates in IL-1 and TLR pathways and thus Pellino proteins have been implicated in these signalling cascades. However the recent identification of Pellino1 as an E3 ubiquitin ligase for RIP1 suggested to us that Pellino proteins may be able to regulate TNF signalling. While the role of Pellino1 in TNF signalling was not explored in Peli1-deficient mice [37] , earlier studies using gene knockdown technology in cell lines reported that Pellino1 and Pellino2 don’t have a role in TNF-induced activation of NF-κB [44] , [45] . Here we explore the role of Pellino3 in TNF signalling. We now demonstrate that Pellino3 has an important regulatory role in the TNF signalling pathway. Knockdown or genetic deficiency of Pellino3 sensitizes cell to TNF-induced apoptosis without inhibiting activation of NF-κB. Instead, loss of Pellino3 leads to increased complex II formation in response to TNF and we show that Pellino3 can normally regulate TNF-induced complex II generation and caspase 8-mediated cleavage of RIP1 by targeting RIP1 in a manner that is dependent on the FHA domain but independent of the RING-like domain of Pellino3. Pellino3-deficient mice also show greatly increased sensitivity to TNF-induced hepatotoxicity and ultimately lethality, thus emphasizing a physiological role of Pellino3 in determining cell fate in response to TNF challenge. Knockdown of Pellino3 enhances pro-apoptotic effects of TNF Previous reports had indicated that Pellino1 and Pellino2 don’t have a role in TNF signalling [44] , [45] but the lack of any data exploring the role of Pellino3 in the TNF pathway prompted the present study. We initially used the Hela cell system in conjunction with Pellino3-specific shRNA to assess the effects of Pellino3 knockdown on TNF-induced apoptosis. TNF is well known to cause cell death in the presence of protein synthesis inhibitors by virtue of the latter preventing the induction of anti-apoptotic proteins. Thus, the combined treatment of Hela cells with TNF and cycloheximide caused the cells to become rounded and non-adherent but the number of such cells was greatly increased when Pellino3 expression was suppressed by Pellino3-specific shRNA ( Fig. 1a ). A MTT-based viability assay revealed that these morphological changes were associated with reduced cell viability in response to TNF and cycloheximide ( Fig. 1b ). Such decreased viability was due to increased apoptosis, because knockdown of Pellino3 expression caused greatly enhanced annexin V staining of Hela cells when co-treated with TNF and cycloheximide and this increased staining was not apparent when cells were treated with the caspase inhibitor ZVAD ( Fig. 1c ). Furthermore, reduced Pellino3 expression also led to an increased cleavage of PARP, caspase 3 and caspase 8 in response to the co-treatment ( Fig. 1d ). These molecular apoptotic signatures add further support to our contention that Pellino3 knockdown sensitizes cells to the pro-apoptotic effects of TNF/cycloheximide. The suppression of Pellino3 expression also enhanced the pro-apoptotic effects of TNF alone, in the absence of cycloheximide, as demonstrated by increased cell detachment ( Supplementary Fig. S1a ) and PARP and caspase 3 cleavage ( Supplementary Fig. S1b ) in Pellino3 knockdown Hela cells treated with TNF alone. In order to assess if the pro-apoptotic effects of suppressed Pellino3 expression were cell-type-dependent similar studies were performed in a human astrocytoma cell line 1321N1. The same effects were apparent in that suppression of Pellino3 expression in 1321N1 cells enhanced the capacity of TNF and cycloheximide to cause cell detachment and rounding ( Supplementary Fig. S1c ), reduce viability ( Supplementary Fig. S1d ) and promote PARP, caspase 3 and caspase 8 cleavage ( Supplementary Fig. S1e ). We next assessed if Pellino3 knockdown had any effects on the ability of TNF to activate the NF-κB or p38 and JNK MAP kinase signalling pathways. The suppression of Pellino3 in 1321N1 cells failed to regulate the ability of TNF to promote degradation of the NF-κB inhibitory protein, IκBα or induce activation of p38 or JNK MAPK ( Supplementary Fig. S1f ). Given the apparent lack of role for Pellino3 in these pathways, Pellino3 was next assessed for its potential to directly regulate complex II formation in response to TNF/cycloheximide. Using co-immunoprecipitation studies on the endogenous signalling proteins we confirmed previous reports that TNF promotes time-dependent interaction of caspase 8 with FADD and RIP1 to form complex II in Hela cells ( Fig. 1e ). However suppressed expression of Pellino3, using Pellino3-specific shRNA constructs, resulted in greater levels of RIP1 and FADD interacting with caspase 8 and such increased complex II formation is consistent with the greater pro-apoptotic effects of TNF/cycloheximide in cells where Pellino3 expression is suppressed. 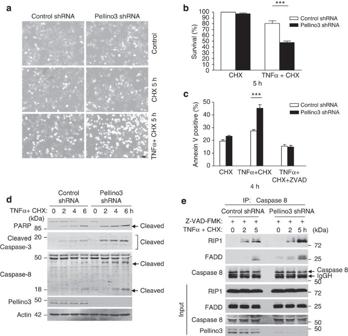Figure 1: Pellino3 knockdown sensitizes Hela cells to TNF/cycloheximide-induced apoptosis. (a–e) Hela cells were infected with lentivirus containing constructs that encoded control or human Pellino3-specific shRNA. Cells were grown in the presence of puromycin to select for cells showing stable integration of shRNA constructs. Selected cells were treated in the absence (control) or presence of human TNF (40 ng ml−1), cycloheximide (CHX) (10 μg ml−1) or the caspase inhibitor benzyloxycarbonyl-valine-alanine-aspartate-fluoromethyl ketone (ZVAD) (20 μM) for 5 h or other indicated times. (a) Cells were photographed using a phase contrast microscope (bar 20 μm). (b) Cells were analysed for cell viability using MTT assays with viability expressed relative to control shRNA-infected cells treated with CHX alone. ***P<0.001 (two-way ANOVA). (c) Cells were analysed by flow cytometry for percentage of cells staining positive for annexin V staining. Data represent the mean +/− s.e.m. of three independent experiments; ***P<0.001 (two-way ANOVA). (d) Cell lysates were probed by immunoblotting for expression levels of PARP, caspase 3, caspase 8, Pellino3 and β-actin. Cleaved forms of PARP and caspase 8 are indicated by arrows. (e) In addition to the indicated treatments all cells were treated with ZVAD to prevent activation of caspase 8 and cell death. Cell lysates were immunoprecipitated with an anti-caspase 8 antibody and immunoprecipitates were subsequently analysed for co-precipitated RIP1, FADD and caspase 8 by western blotting. The expression levels of RIP1, FADD, caspase 8 and Pellino3 in whole-cell lysates (‘input’) were also assessed by western blotting. Full-length images of immunoblots are shown inSupplementary Fig. S8. Figure 1: Pellino3 knockdown sensitizes Hela cells to TNF/cycloheximide-induced apoptosis. ( a – e ) Hela cells were infected with lentivirus containing constructs that encoded control or human Pellino3-specific shRNA. Cells were grown in the presence of puromycin to select for cells showing stable integration of shRNA constructs. Selected cells were treated in the absence (control) or presence of human TNF (40 ng ml −1 ), cycloheximide (CHX) (10 μg ml −1 ) or the caspase inhibitor benzyloxycarbonyl-valine-alanine-aspartate-fluoromethyl ketone (ZVAD) (20 μM) for 5 h or other indicated times. ( a ) Cells were photographed using a phase contrast microscope (bar 20 μm). ( b ) Cells were analysed for cell viability using MTT assays with viability expressed relative to control shRNA-infected cells treated with CHX alone. *** P <0.001 (two-way ANOVA). ( c ) Cells were analysed by flow cytometry for percentage of cells staining positive for annexin V staining. Data represent the mean +/− s.e.m. of three independent experiments; *** P <0.001 (two-way ANOVA). ( d ) Cell lysates were probed by immunoblotting for expression levels of PARP, caspase 3, caspase 8, Pellino3 and β-actin. Cleaved forms of PARP and caspase 8 are indicated by arrows. ( e ) In addition to the indicated treatments all cells were treated with ZVAD to prevent activation of caspase 8 and cell death. Cell lysates were immunoprecipitated with an anti-caspase 8 antibody and immunoprecipitates were subsequently analysed for co-precipitated RIP1, FADD and caspase 8 by western blotting. The expression levels of RIP1, FADD, caspase 8 and Pellino3 in whole-cell lysates (‘input’) were also assessed by western blotting. Full-length images of immunoblots are shown in Supplementary Fig. S8 . Full size image To further validate the above conclusion that Pellino3 knockdown enhanced TNF-induced apoptosis we used HEK293 cells to demonstrate that the independent approaches of employing shRNA expression constructs or synthesized siRNAs to suppress Pellino3 expression manifested the same findings in terms of increasing sensitivity of cells to the pro-apoptotic effects of TNF. Thus, as was the case with Hela and 1321N1 cells, Pellino3-specific shRNA increased annexin V staining of HEK293 cells in response to TNF/cycloheximide and this could be blocked with the caspase inhibitor ZVAD ( Fig. 2a ). In addition these cells demonstrated increased levels of cleaved PARP, caspase 3 and caspase 8 in response to TNF/cycloheximide ( Fig. 2b ). Furthermore, the knockdown of Pellino3 in HEK293 cells, using Pellino3-specific siRNA that targets a different region of the Pellino3 mRNA, also enhanced the pro-apoptotic effects of TNF alone as evidenced by greater levels of cleaved PARP, caspase 3 and caspase 8 ( Supplementary Fig. S2a ), increased TUNEL staining ( Supplementary Fig. S2b ) and enhanced complex II formation ( Supplementary Fig. S2c ). These findings, employing independent approaches to suppress Pellino3 expression in different cell lines, provide strong evidence that Pellino3 has a key role in regulating complex II formation and apoptosis in response to TNF. 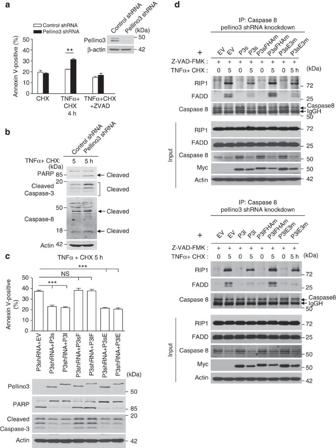Figure 2: Pellino3 regulates TNF-induced apoptosis in a FHA-dependent but RING-like domain-independent manner. (a,b) HEK293 cells were infected with lentivirus containing control or Pellino3-specific shRNA and treated with human TNF (50 ng ml−1), cycloheximide (CHX) (10 μg ml−1) or the caspase inhibitor ZVAD (20 μM). (a) Cells were analysed by flow cytometry for annexin V staining (mean +/− s.e.m. of three independent experiments; **P<0.01; two-way ANOVA). Immunoblot analysis demonstrating Pellino3 protein knockdown. (b) Cell lysates were immunoblotted for PARP, caspase 3, caspase 8 and β-actin. Cleaved forms of PARP and caspase 8 are indicated by arrows. (c,d) HEK293 cells, previously transfected with an expression construct encoding Pellino3-specific shRNA, were transfected with pcDNA3.1 empty vector (EV) or pcDNA3.1 encoding myc-tagged Pellino3s, Pellino3l, Pellino3s(R131A/S161A)-myc (Pellino3sFHAm), Pellino3l(R155A/S185A)-myc (Pellino3lFHAm), Pellino3s(C360A/C363 A)-myc (Pellino3sE3m) and Pellino3l (C384A/C387A)-myc (Pellino3lE3m). (c) Transfected cells were treated with human TNF (40 ng ml−1) and cycloheximide (CHX) (10 μg ml−1) for 5 h and analysed by flow cytometry for percentage of cells staining positive for annexin V staining. Data represent the mean +/− s.e.m. of three independent experiments; ***P<0.001 (two-way ANOVA). The expression levels of Pellino3, PARP, cleaved caspase 3 and β-actin were measured in cell lysates by western blotting. (d) In addition to the indicated treatments with TNF and cycloheximide (above) cells were also treated with ZVAD to prevent activation of caspase 8 and cell death. Cell lysates were immunoprecipitated with an anti-caspase 8 antibody and immunoprecipitates were subsequently analysed for co-precipitated RIP1, FADD and caspase 8 by western blotting. The expression levels of RIP1, FADD, caspase 8, Pellino3 and β-actin were measured in whole-cell lysates (‘input’) by western blotting. Full-length images of immunoblots are shown inSupplementary Fig. S9. Figure 2: Pellino3 regulates TNF-induced apoptosis in a FHA-dependent but RING-like domain-independent manner. ( a , b ) HEK293 cells were infected with lentivirus containing control or Pellino3-specific shRNA and treated with human TNF (50 ng ml −1 ), cycloheximide (CHX) (10 μg ml −1 ) or the caspase inhibitor ZVAD (20 μM). ( a ) Cells were analysed by flow cytometry for annexin V staining (mean +/− s.e.m. of three independent experiments; ** P <0.01; two-way ANOVA). Immunoblot analysis demonstrating Pellino3 protein knockdown. ( b ) Cell lysates were immunoblotted for PARP, caspase 3, caspase 8 and β-actin. Cleaved forms of PARP and caspase 8 are indicated by arrows. ( c , d ) HEK293 cells, previously transfected with an expression construct encoding Pellino3-specific shRNA, were transfected with pcDNA3.1 empty vector (EV) or pcDNA3.1 encoding myc-tagged Pellino3s, Pellino3l, Pellino3s(R131A/S161A)-myc (Pellino3sFHAm), Pellino3l(R155A/S185A)-myc (Pellino3lFHAm), Pellino3s(C360A/ C 363 A)-myc (Pellino3sE3m) and Pellino3l (C384A/C387A)-myc (Pellino3lE3m). ( c ) Transfected cells were treated with human TNF (40 ng ml −1 ) and cycloheximide (CHX) (10 μg ml −1 ) for 5 h and analysed by flow cytometry for percentage of cells staining positive for annexin V staining. Data represent the mean +/− s.e.m. of three independent experiments; *** P <0.001 (two-way ANOVA). The expression levels of Pellino3, PARP, cleaved caspase 3 and β-actin were measured in cell lysates by western blotting. ( d ) In addition to the indicated treatments with TNF and cycloheximide (above) cells were also treated with ZVAD to prevent activation of caspase 8 and cell death. Cell lysates were immunoprecipitated with an anti-caspase 8 antibody and immunoprecipitates were subsequently analysed for co-precipitated RIP1, FADD and caspase 8 by western blotting. The expression levels of RIP1, FADD, caspase 8, Pellino3 and β-actin were measured in whole-cell lysates (‘input’) by western blotting. Full-length images of immunoblots are shown in Supplementary Fig. S9 . Full size image Pellino3 regulates TNF signalling via its FHA domain We next assessed the functional contribution of the different domains of Pellino3 to its regulatory effects on TNF signalling. This was addressed by experiments that aimed to rescue the phenotypic effects of Pellino3 knockdown on TNF signalling in HEK293 cells, using various mutant forms of Pellino. The use of a Pellino3-specific shRNA that targets the 3′ untranslated region (UTR) of the Pellino3 mRNA provided an opportunity to demonstrate that expression constructs encoding either spliced form of Pellino3 but lacking the 3′ UTR could rescue the increased pro-apoptotic effects of TNF that was observed in Pellino3 knockdown cells. Both Pellino3s and Pellino3l prevented the increased annexin V staining and PARP and caspase 3 cleavage that was apparent in knockdown cells ( Fig. 2c ), indicating that both spliced forms can temper the pro-apoptotic signalling of TNF. Furthermore, the mechanistic basis to these effects are due to Pellino3 inhibiting complex II formation in response to TNF/cycloheximide as shown by the ability of both Pellino3s ( Fig. 2d , upper panels) and Pellino3l ( Fig. 2d , lower panels) to rescue the increased interaction of RIP1 and FADD with caspase 8 that was observed in knockdown cells. Using a similar approach we next explored the ability of various mutant forms of Pellino3 ( Supplementary Fig. S3 ) to re-constitute Pellino3 function in Pellino3-deficient cells in order to define the functional relevance of its FHA and RING-like. Forms of Pellino3s and Pellino3l, containing mutations that affect FHA domain structure and function, failed to mimic their wild-type counterparts in inhibiting the TNF/cycloheximide-induced increases in annexinV staining and cleavage of PARP and caspase 3 in Pellino3 knockdown cells ( Fig. 2c ) and furthermore unlike their wild-type forms they failed to inhibit complex II formation in response to TNF ( Fig. 2d ). These findings indicate an important role for the FHA domain of Pellino3 proteins in counter-regulating the pro-apoptotic proclivity of TNF signalling. Pellino proteins also contain a RING-like domain that is associated with E3 ubiquitin ligase activity and we next investigated the importance of this domain for the regulatory effects of Pellino3 on TNF signalling. We thus mutated key cysteine residues in the RING-like domain of Pellino3 that abrogate the E3 ubiquitin ligase activity of wild-type Pellino3 ( Supplementary Fig. S4 ). However, forms of Pellino3s and Pellino3l, containing such mutations in their RING-like domain, inhibited the ability of TNF to promote increased annexin V staining and cleavage of PARP and caspase 3 in Pellino3 knockdown cells ( Fig. 2a ) and like wild-type Pellino3 they also reduced the levels of complex II in response to TNF/cycloheximide ( Fig. 2b ). These data suggest a dispensable role for the RING-like domain and the E3 ligase catalytic activity of Pellino3 in manifesting its regulatory effects on TNF signalling. In contrast, the FHA domain is of crucial importance. Pellino3 targets RIP1 in a FHA domain-dependent manner Given the ability of Pellino3 to regulate TNF-induced complex II formation, we next characterized the ability of Pellino3 to interact with the individual protein components of complex II. We first probed the ability of Pellino3 to interact with RIP1. The co-expression of Pellino3s or 3l with RIP1 leads to their strong interaction as shown by co-immunoprecipitation of Pellino3 and RIP1 ( Fig. 3a ). The FHA mutants of Pellino3 showed considerable diminution in terms of binding to RIP1, supporting a model where the FHA domain of Pellino3 facilitates its interaction with RIP1. Barely detectable levels of purified RIP1 were shown to co-immunoprecipitate with purified recombinant forms of Pellino3s and 3l ( Fig. 3b ), indicating that both forms of Pellino3 can directly interact with RIP1, but with very low efficiency. Purified forms of Pellino3 were more effective in co-precipitating RIP1 from cell lysates ( Fig. 3c ), suggesting that the Pellino3/RIP1 interaction may be enhanced by some modification of RIP1 in cells or its interaction with some ancillary protein(s). Again the purified FHA mutants of Pellino3 were greatly diminished relative to their wild-type equivalents in their interactions with RIP1 ( Fig. 3c ), adding further support to a model in which Pellino3 targets RIP1 in a FHA domain-dependent manner. 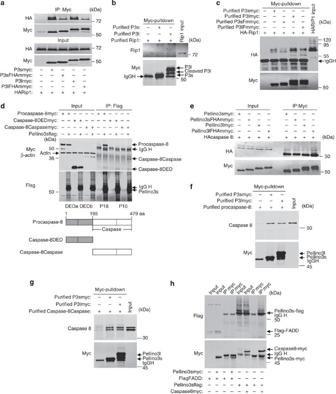Figure 3: Pellino3 interacts with RIP1 and caspase 8 but not FADD. (a) HEK293 cells were co-transfected with indicated constructs encoding HA-tagged RIP1 and myc-tagged Pellino3s or Pellino3l or their corresponding FHA mutants (Pellino3s(R131A/S161A) (Pellino3sFHAm), or Pellino3l(R155A/S185A) (Pellino3lFHAm)). Such transfections also included co-expression of the caspase inhibitor CrmA to prevent caspase-induced cleavage of RIP1 and cell apoptosis. Cell lysates were immunoprecipitated (IP) using an anti-myc antibody followed by immunoblotting using anti-HA or -myc antibodies. Cell lysates, prior to immunoprecipitation (input), were similarly analysed by immunoblotting. (b,c) Purified recombinant myc-tagged Pellino3s, Pellino3l or their FHA mutant counterparts were immunoprecipitated with an anti-myc antibody and then incubated with (b) purified recombinant RIP1 protein or (c) HEK293 cell lysates from cells previously transfected with HA-tagged RIP1. Samples were then precipitated (myc-pulldown) and analysed by immunoblotting using anti-RIP1, -HA or -myc antibodies. Input samples represent purified RIP1 protein (b) or a cell lysate from HEK293 cells previously transfected with HA-tagged RIP1 (c). (d) HEK293 cells were co-transfected with the indicated constructs encoding myc-tagged procaspase 8, caspase 8 DED domain (residues 1–194), caspase 8-caspase domain (residues 195–479) and flag-tagged Pellino3s. Cell lysates were immunoprecipitated (IP) using an anti-flag antibody followed by immunoblotting (IB) using anti-myc, -flag or –βactin antibodies. Cell lysates, prior to immunoprecipitation (Input), were similarly analysed by immunoblotting. (e) HEK293 cells were co-transfected with indicated combinations of constructs encoding HA-tagged procaspase 8 and myc-tagged Pellino3s or Pellino3l or their corresponding FHA mutants as described above. Cell lysates were immunoprecipitated (IP) using an anti-myc antibody followed by immunoblotting using anti-HA or -myc antibodies. Cell lysates, prior to immunoprecipitation (input), were similarly analysed by immunoblotting. (f,g) Purified myc-tagged Pellino3s or Pellino3l was immunoprecipitated with anti-myc antibody and then incubated with purified (f) procaspase 8 protein or (g) caspase 8-caspase domain. Samples were then precipitated (myc-pulldown) and analysed by immunoblotting using anti-myc or –caspase 8 antibodies. Samples of recombinant Pellino proteins, procaspase 8 and caspase 8-caspase domain (Input) were similarly analysed by immunoblotting. (h) HEK293 cells were co-transfected with constructs expressing myc-tagged Pellino3s and/or Flag-tagged FADD. Cell lysates were immunoprecipitated (IP) using an anti-myc antibody followed by immunoblotting using anti-Flag or -myc antibodies. Cell lysates, prior to immunoprecipitation (input), were similarly analysed by immunoblotting. Full-length images of immunoblots are shown inSupplementary Fig. S10. Figure 3: Pellino3 interacts with RIP1 and caspase 8 but not FADD. ( a ) HEK293 cells were co-transfected with indicated constructs encoding HA-tagged RIP1 and myc-tagged Pellino3s or Pellino3l or their corresponding FHA mutants (Pellino3s(R131A/S161A) (Pellino3sFHAm), or Pellino3l(R155A/S185A) (Pellino3lFHAm)). Such transfections also included co-expression of the caspase inhibitor CrmA to prevent caspase-induced cleavage of RIP1 and cell apoptosis. Cell lysates were immunoprecipitated (IP) using an anti-myc antibody followed by immunoblotting using anti-HA or -myc antibodies. Cell lysates, prior to immunoprecipitation (input), were similarly analysed by immunoblotting. ( b , c ) Purified recombinant myc-tagged Pellino3s, Pellino3l or their FHA mutant counterparts were immunoprecipitated with an anti-myc antibody and then incubated with ( b ) purified recombinant RIP1 protein or ( c ) HEK293 cell lysates from cells previously transfected with HA-tagged RIP1. Samples were then precipitated (myc-pulldown) and analysed by immunoblotting using anti-RIP1, -HA or -myc antibodies. Input samples represent purified RIP1 protein ( b ) or a cell lysate from HEK293 cells previously transfected with HA-tagged RIP1 ( c ). ( d ) HEK293 cells were co-transfected with the indicated constructs encoding myc-tagged procaspase 8, caspase 8 DED domain (residues 1–194), caspase 8-caspase domain (residues 195–479) and flag-tagged Pellino3s. Cell lysates were immunoprecipitated (IP) using an anti-flag antibody followed by immunoblotting (IB) using anti-myc, -flag or –βactin antibodies. Cell lysates, prior to immunoprecipitation (Input), were similarly analysed by immunoblotting. ( e ) HEK293 cells were co-transfected with indicated combinations of constructs encoding HA-tagged procaspase 8 and myc-tagged Pellino3s or Pellino3l or their corresponding FHA mutants as described above. Cell lysates were immunoprecipitated (IP) using an anti-myc antibody followed by immunoblotting using anti-HA or -myc antibodies. Cell lysates, prior to immunoprecipitation (input), were similarly analysed by immunoblotting. ( f , g ) Purified myc-tagged Pellino3s or Pellino3l was immunoprecipitated with anti-myc antibody and then incubated with purified ( f ) procaspase 8 protein or ( g ) caspase 8-caspase domain. Samples were then precipitated (myc-pulldown) and analysed by immunoblotting using anti-myc or –caspase 8 antibodies. Samples of recombinant Pellino proteins, procaspase 8 and caspase 8-caspase domain (Input) were similarly analysed by immunoblotting. ( h ) HEK293 cells were co-transfected with constructs expressing myc-tagged Pellino3s and/or Flag-tagged FADD. Cell lysates were immunoprecipitated (IP) using an anti-myc antibody followed by immunoblotting using anti-Flag or -myc antibodies. Cell lysates, prior to immunoprecipitation (input), were similarly analysed by immunoblotting. Full-length images of immunoblots are shown in Supplementary Fig. S10 . Full size image Pellino3 was next assessed for its ability to interact with caspase 8, another key component of complex II. The co-expression of procaspase 8 (with a C360A mutation to prevent autocleavage) with Pellino3s followed by co-immunoprecipitation analysis demonstrated that both proteins co-precipitate with each other ( Fig. 3d ). Interestingly, the interaction of Pellino3 with procaspase 8 in co-expression studies is independent of the FHA domain of the former because FHA mutants of Pellino3s and Pellino3l mimicked their wild-type counterparts in co-immunoprecipitating with procaspase 8 ( Fig. 3e ). We also show that the interaction between Pellino3 and procaspase 8 is direct in nature, as purified recombinant forms of both proteins interact with each other in vitro ( Fig. 3f ). We next characterized the regions of procaspase 8 that mediate binding to Pellino3. Procaspase 8 contains two death effector domains (DEDa and DEDb) in its N-terminal pro-domain and a C-terminal region that encodes for the catalytic large (p18) and small subunits (p10). Expression constructs encoding procaspase 8, DEDa/DEDb and caspase regions of caspase 8 were co-expressed with Pellino3s. Co-immunoprecipitation analysis showed that procaspase 8 and its caspase region interacted with Pellino3, whereas there was no such interaction between the DEDa/DEDb domain of procaspase 8 and Pellino3 ( Fig. 3d ). Furthermore, the interaction of the caspase domain with Pellino3 was proven to be direct in nature by showing that a purified recombinant form of the caspase domain interacts with purified Pellino3s and Pellino3l in an in vitro binding assay ( Fig. 3g ). These findings thus indicate that Pellino3 can interact with RIP1 in a FHA domain-dependent manner, whereas the latter domain is not used by Pellino3 in its direct targeting of the caspase domain of procaspase 8. We also generated a truncation mutant (encoding residues 1-313) of Pellino3s, termed Pellino3sΔC(1–313aa) that lacked the C-terminal RING-like domain and predominantly consisted of the N-terminal FHA domain. This mutant was shown to retain the ability of its full-length counterpart to bind to RIP1, as evidenced by reciprocal co-immunoprecipitation of RIP1 and Pellino3sΔC, whereas it failed to interact with caspase 8 ( Supplementary Fig. S5a,b ). These findings indicate that the FHA domain of Pellino3 provides sufficient structure to physically interact with RIP1, whereas it is fails to provide the required structure for association with caspase 8. We finally investigated the ability of Pellino3 to interact with FADD, another critical constituent of complex II. However co-expression studies failed to show an association of Pellino3 with FADD ( Fig. 3h ). The interaction of Pellino3 with caspase 8 was used as a positive control. The dynamics of the interactions between endogenous Pellino3 and RIP1 and caspase 8 in response to TNF were next addressed. Cells were treated with TNF, cycloheximide and the caspase inhibitor ZVAD to block any RIP1 processing. RIP1 was immunoprecipitated and assessed for co-precipitated levels of Pellino3 and the complex II components, caspase 8 and FADD. Using this approach TNF was shown to promote complex II formation as evidenced by time-dependent binding of RIP1 to caspase 8 and FADD ( Fig. 4a ). Interestingly, this was also accompanied by TNF-induced association of RIP1 with both spliced forms of Pellino3. In parallel experiments, endogenous caspase 8 was immunoprecipitated and probed for the presence of co-precipitated Pellino3, RIP1 and FADD. Complex II was again formed in response to TNF/cycloheximide, as demonstrated by time-dependent interaction of caspase 8 with RIP1 and FADD ( Fig. 4b ). Interestingly, Pellino3 was associated with caspase 8 in unstimulated cells but the interaction was not regulated by TNF. These studies suggest that Pellino3 basally interacts with caspase 8 and associates with RIP1 in response to TNF stimulation to regulate complex II formation. However, given that RIP1 is also a part of complex I that forms in response TNF stimulation we investigated if TNF could promote the recruitment of Pellino3 to complex I. Hela cells were thus stimulated with TNF alone for shorter times to study complex I formation, after which TNFRI was immunoprecipitated and probed for complex I components. TNF caused a time-dependent formation of complex I as judged by the interaction of TNFRI with RIP1 and TRAF2 ( Fig. 4c ). However, Pellino3 was not recruited to TNFRI at these early times suggesting that Pellino3 is not part of complex I in the TNF pathway. Instead TNF promotes the binding of Pellino3 to RIP1 to counter-regulate the formation of complex II. 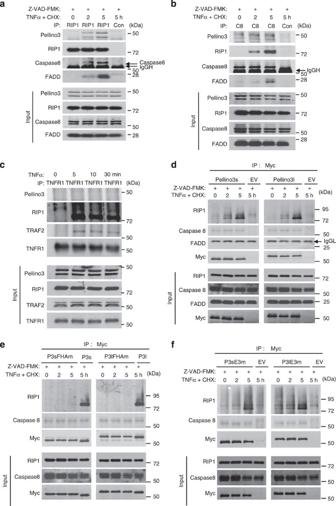Figure 4: TNF promotes binding of Pellino3 to RIP1 in a FHA domain-dependent manner but not as part of complex I. (a,b) Hela cells were treated in the absence or presence of TNF (50 ng ml−1) and cycloheximide (CHX) (10 μg ml−1) for the indicated times. Cells were also treated with the pan-caspase inhibitor ZVAD (20 μM) to prevent full activation of caspase 8 and cell death. Cell lysates were immunoprecipitated with anti-RIP1 (a) or anti-caspase 8 (b) antibodies. Mouse IgG and goat IgG were used for respective control immunoprecipitations. The immunoprecipitates were subsequently analysed for co-precipitated Pellino3, RIP1, caspase 8 and FADD by western blotting. The expression levels of Pellino3, RIP1, caspase 8 and FADD proteins were measured in whole-cell lysates (input) by western blotting. The precipitated IgG heavy chain (IgGH) is also indicated by an arrow. (c) Hela cells were treated in the absence or presence of TNF (50 ng ml−1) for indicated times. Cell lysates were immunoprecipitated with anti-TNFR1 antibody. The immunoprecipitates were subsequently analysed for co-precipitated Pellino3, RIP1, TRAF2 and TNFR1 by western blotting. The expression levels of Pellino3, RIP1, TRAF2 and TNFR1 proteins were measured in whole-cell lysates (input) by western blotting. (d–f) HEK293 cells were transfected with an empty vector (EV) or expression constructs encoding (d) myc-taggged Pellino3s or Pellino3l, (e) FHA domain mutant forms of Pellino3s(R131A/S161A) (Pellino3sFHAm) or Pellino3l(R155A/S185A) (Pellino3lFHAm) or (f) RING-like domain mutant forms of Pellino3s (C360A/C363A) (Pellino3sE3m) and Pellino3l (C384A/C387A) (Pellino3lE3m). Cells were then treated in the absence or presence of TNF (50 ng ml−1) and cycloheximide (CHX) (10 μg ml−1) for indicated times. Cells were also treated with the pan-caspase inhibitor ZVAD (20 μM) to prevent full activation of caspase 8 and cell death. Cell lysates were immunoprecipitated with an anti-myc antibody and immunoprecipitates were subsequently analysed for co-precipitated RIP1, caspase 8, FADD and myc-tagged Pellino proteins by western blotting. The precipitated IgG light chain (IgGL) is indicated by an arrow. The expression levels of RIP1, caspase 8, FADD and myc-tagged Pellino proteins were measured in whole-cell lysates (input) by western blotting. Full-length images of immunoblots are shown inSupplementary Fig. S11. Figure 4: TNF promotes binding of Pellino3 to RIP1 in a FHA domain-dependent manner but not as part of complex I. ( a , b ) Hela cells were treated in the absence or presence of TNF (50 ng ml −1 ) and cycloheximide (CHX) (10 μg ml −1 ) for the indicated times. Cells were also treated with the pan-caspase inhibitor ZVAD (20 μM) to prevent full activation of caspase 8 and cell death. Cell lysates were immunoprecipitated with anti-RIP1 ( a ) or anti-caspase 8 ( b ) antibodies. Mouse IgG and goat IgG were used for respective control immunoprecipitations. The immunoprecipitates were subsequently analysed for co-precipitated Pellino3, RIP1, caspase 8 and FADD by western blotting. The expression levels of Pellino3, RIP1, caspase 8 and FADD proteins were measured in whole-cell lysates (input) by western blotting. The precipitated IgG heavy chain (IgGH) is also indicated by an arrow. ( c ) Hela cells were treated in the absence or presence of TNF (50 ng ml −1 ) for indicated times. Cell lysates were immunoprecipitated with anti-TNFR1 antibody. The immunoprecipitates were subsequently analysed for co-precipitated Pellino3, RIP1, TRAF2 and TNFR1 by western blotting. The expression levels of Pellino3, RIP1, TRAF2 and TNFR1 proteins were measured in whole-cell lysates (input) by western blotting. ( d – f ) HEK293 cells were transfected with an empty vector (EV) or expression constructs encoding ( d ) myc-taggged Pellino3s or Pellino3l, ( e ) FHA domain mutant forms of Pellino3s(R131A/S161A) (Pellino3sFHAm) or Pellino3l(R155A/S185A) (Pellino3lFHAm) or ( f ) RING-like domain mutant forms of Pellino3s (C360A/C363A) (Pellino3sE3m) and Pellino3l (C384A/C387A) (Pellino3lE3m). Cells were then treated in the absence or presence of TNF (50 ng ml −1 ) and cycloheximide (CHX) (10 μg ml −1 ) for indicated times. Cells were also treated with the pan-caspase inhibitor ZVAD (20 μM) to prevent full activation of caspase 8 and cell death. Cell lysates were immunoprecipitated with an anti-myc antibody and immunoprecipitates were subsequently analysed for co-precipitated RIP1, caspase 8, FADD and myc-tagged Pellino proteins by western blotting. The precipitated IgG light chain (IgGL) is indicated by an arrow. The expression levels of RIP1, caspase 8, FADD and myc-tagged Pellino proteins were measured in whole-cell lysates (input) by western blotting. Full-length images of immunoblots are shown in Supplementary Fig. S11 . Full size image We next investigated the importance of the FHA and RING-like domains of Pellino3 for mediating its interactions with RIP1 and caspase 8 in the context of TNF signalling. This was achieved by expressing wild-type and mutant forms (mutated FHA and RING-like domains) of Pellino3s and Pellino3l in HEK293 cells and characterizing their interaction with RIP1 and caspase 8 in response to TNF/cycloheximide stimulation. Co-immunoprecipitation analyses demonstrated that TNF promoted a strong and time-dependent interaction between endogenous RIP1 and Pellino3s ( Fig. 4d ; left panels) or Pellino3l ( Fig. 4d ; right panels). Again both forms of Pellino3 interacted with endogenous caspase 8 in unstimulated cells and treatment with TNF failed to further enhance this interaction ( Fig. 4d ). Furthermore, neither form of Pellino3 showed association with FADD irrespective of the absence or presence of TNF. Mutations in the FHA domain of either form of Pellino3 abrogated the ability of the latter to interact with RIP1, even in the presence of TNF stimulus ( Fig. 4e ). Interestingly, the FHA mutants retained the capacity to interact with caspase 8, suggesting a selective role for the FHA domain in the targeting of RIP1. Given also the important role for the FHA domain in facilitating the regulatory effects of Pellino3 on TNF signalling these data suggest that the targeting of RIP1 by Pellino3 is of likely importance in its functional modulation of the TNF pathway. In contrast, the introduction of mutations in the RING-like domain of Pellino3s and Pellino3l failed to affect their associations with RIP1 or caspase 8 ( Fig. 4f ), excluding a role for this domain in facilitating such interactions. This is consistent with the lack of importance of the RING-like domain in mediating the regulatory effects of Pellino3 on TNF signalling. We next hypothesized that the targeting of RIP1 by Pellino3 may interfere with the recruitment of RIP1 to the caspase 8/FADD complex. In support of this hypothesis we detected greater levels of RIP1-associated FADD in Pellino3 knockdown cells ( Supplementary Fig. S2d ) and conversely overexpression of Pellino3s significantly diminished the levels of FADD and caspase 8 that co-immunoprecipitated with RIP1 in extracts from TNF/cycloheximide-stimulated HEK293 cells ( Fig. 5 ). In contrast, overexpression of a FHA mutant form of Pellino3 failed to affect the recruitment of FADD and caspase 8 to RIP1, whereas the RING-like domain mutant form of Pellino3s mimicked the inhibitory effects of its wild-type counterpart ( Fig. 5 ). These findings further support our model that Pellino3 targets RIP1 in a FHA domain-dependent manner, thus preventing its recruitment of FADD and caspase 8. Interestingly, Pellino3sΔC, that primarily consists of the FHA domain and can interact with RIP1 but not caspase 8 failed to regulate the association of FADD and caspase 8 with RIP1 ( Fig. 5 ), suggesting that the binding of Pellino3 to RIP1, via its FHA domain, is required but not sufficient to regulate the recruitment of RIP1 to the caspase 8/FADD complex. 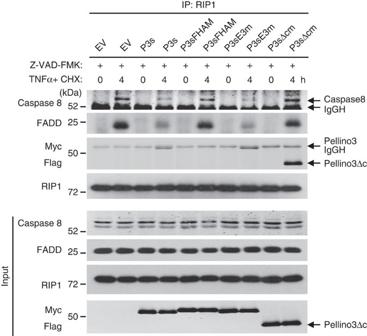Figure 5: Pellino3 inhibits formation of Complex II in a FHA-dependent but RING-like domain-independent manner. HEK293 cells were transfected with pcDNA3.1 empty vector (EV) or pcDNA3.1 encoding myc-tagged Pellino3s (P3s), Pellino3s(R131A/S161A)-myc (P3sFHAm), Pellino3s(C360A/C363A)-myc (P3sE3m) and flag-Pellino3sΔC(1–313aa) (P3sΔcm). Transfected cells were treated with human TNF (40 ng ml−1), cycloheximide (CHX) (10 μg ml−1) and ZVAD(20 μM) for 4 h. Cell lysates were immunoprecipitated with an anti-RIP1 antibody and immunoprecipitates were subsequently analysed for co-precipitated RIP1, FADD, Myc, Flag and caspase 8 by western blotting. The expression levels of RIP1, FADD, caspase 8 and Pellino3 were measured in whole-cell lysates (input) by western blotting. Full-length images of immunoblots are shown inSupplementary Fig. S12. Figure 5: Pellino3 inhibits formation of Complex II in a FHA-dependent but RING-like domain-independent manner. HEK293 cells were transfected with pcDNA3.1 empty vector (EV) or pcDNA3.1 encoding myc-tagged Pellino3s (P3s), Pellino3s(R131A/S161A)-myc (P3sFHAm), Pellino3s(C360A/C363A)-myc (P3sE3m) and flag-Pellino3sΔC(1–313aa) (P3sΔcm). Transfected cells were treated with human TNF (40 ng ml −1 ), cycloheximide (CHX) (10 μg ml −1 ) and ZVAD(20 μM) for 4 h. Cell lysates were immunoprecipitated with an anti-RIP1 antibody and immunoprecipitates were subsequently analysed for co-precipitated RIP1, FADD, Myc, Flag and caspase 8 by western blotting. The expression levels of RIP1, FADD, caspase 8 and Pellino3 were measured in whole-cell lysates (input) by western blotting. Full-length images of immunoblots are shown in Supplementary Fig. S12 . Full size image Enhanced TNF-induced apoptosis in Pellino3-deficient cells In order to define the physiological relevance of the role of Pellino3 in TNF signalling, Pellino3-deficient mice were used. Mice were generated as previously described [46] . Murine embryonic fibroblasts (MEFs) from Pellino3 +/+ and Pellino3 −/− mice were initially used to assess the effects of Pellino3 deficiency on TNF signalling. Co-stimulation of MEFs with TNF and cycloheximide caused the cells to become rounded and non-adherent but such phenotypic changes were much more apparent in MEFs from Pellino3 −/− embryos relative to their wild-type control cells ( Fig. 6a ). These changes were associated with greater levels of apoptosis as revealed by more annexin V staining ( Fig. 6b ) and greater levels of cleaved PARP and caspase 3 ( Fig. 6c ) in cells from Pellino3 −/− mice. This increased apoptotic susceptibility of Pellino3-deficient cells appears to be specific for TNF as a death signal because MEFs from Pellino3 −/− embryos do not show any enhanced sensitivity to other pro-apoptotic pathways such as Fas ( Supplementary Fig. S6a,b ) or the gentoxic compound etoposide ( Supplementary Fig. S6c,d ), as measured by annexin V staining ( Supplementary Fig. S6a,c ) and cleavage of PARP and caspase 3 ( Supplementary Fig. S6b,d ). 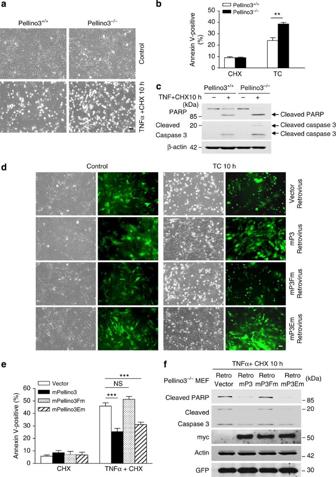Figure 6: Pellino3-deficient MEFs show increased apoptosis in response to TNF/cycloheximide co-stimulation. (a–c) MEFs were isolated from Pellino3+/+and Pellino3−/−embryos and treated in the absence (control) or presence of murine TNF (40 ng ml−1) and cycloheximide (CHX) (10 μg ml−1) for 10 h. (a) Cells were photographed using a phase contrast microscope (bar 20 μm). (b) Cells were analysed by flow cytometry for percentage of cells staining positive for annexin V. Data represent the mean +/− s.e.m. of three independent experiments; **P<0.01 (two-way ANOVA). (c) Cell lysates were probed by immunoblotting for expression levels of PARP, cleaved caspase 3 and β-actin. (d–f) MEFs, from Pellino3−/−embryos, were infected with murine stem cell virus (MSCV), lacking (vector) or containing the myc-tagged murinePellino3gene (mP3 retrovirus), FHA domain mutant form of mPellino3 (mP3Fm) or RING-like domain mutant form of mPellino3 (mP3Em). Infected cells were treated in the absence (control) or presence of murine TNF (40 ng ml−1) and cycloheximide (CHX) (10 μg ml−1) for 10 h. (d) Cells were photographed using a phase contrast microscope (bar 20 μm) or viewed by fluorescent microscopy to detect infected cells based on expression of MSCV-encoded GFP. (e) Cells were analysed by flow cytometry for percentage of cells staining positive for annexin V staining. Data represent the mean +/− s.e.m. of three independent experiments; ***P<0.001; n.s: not significant (two-way ANOVA). (f) Cell lysates were probed by immunoblotting for expression levels of PARP, cleaved caspase 3, myc-Pellino3, β-actin and GFP. Full-length images of immunoblots are shown inSupplementary Fig. S13. Figure 6: Pellino3-deficient MEFs show increased apoptosis in response to TNF/cycloheximide co-stimulation. ( a – c ) MEFs were isolated from Pellino3 +/+ and Pellino3 −/− embryos and treated in the absence (control) or presence of murine TNF (40 ng ml −1 ) and cycloheximide (CHX) (10 μg ml −1 ) for 10 h. ( a ) Cells were photographed using a phase contrast microscope (bar 20 μm). ( b ) Cells were analysed by flow cytometry for percentage of cells staining positive for annexin V. Data represent the mean +/− s.e.m. of three independent experiments; ** P <0.01 (two-way ANOVA). ( c ) Cell lysates were probed by immunoblotting for expression levels of PARP, cleaved caspase 3 and β-actin. ( d – f ) MEFs, from Pellino3 −/− embryos, were infected with murine stem cell virus (MSCV), lacking (vector) or containing the myc-tagged murine Pellino3 gene (mP3 retrovirus), FHA domain mutant form of mPellino3 (mP3Fm) or RING-like domain mutant form of mPellino3 (mP3Em). Infected cells were treated in the absence (control) or presence of murine TNF (40 ng ml −1 ) and cycloheximide (CHX) (10 μg ml −1 ) for 10 h. ( d ) Cells were photographed using a phase contrast microscope (bar 20 μm) or viewed by fluorescent microscopy to detect infected cells based on expression of MSCV-encoded GFP. ( e ) Cells were analysed by flow cytometry for percentage of cells staining positive for annexin V staining. Data represent the mean +/− s.e.m. of three independent experiments; *** P <0.001; n.s: not significant (two-way ANOVA). ( f ) Cell lysates were probed by immunoblotting for expression levels of PARP, cleaved caspase 3, myc-Pellino3, β-actin and GFP. Full-length images of immunoblots are shown in Supplementary Fig. S13 . Full size image In order to ensure that the greater pro-apoptotic effects of TNF in Pellino3 −/− cells were due specifically to Pellino3 deficiency, Pellino3 −/− MEFs were re-constituted with a murine Pellino3 (mPellino3) expression construct using retroviral-mediated transduction. High-efficiency transduction of the cells was confirmed by microscopic detection of co-expressed GFP. Transduction of Pellino3-deficient MEFs with retrovirus containing the murine Pellino3 gene greatly reduced the level of cell detachment and rounding in response to TNF/cycloheximide stimulation ( Fig. 6d ). Furthermore, reconstitution of Pellino3-deficient MEFs with mPellino3 significantly reduced annexin V staining in response to TNF/cycloheximide ( Fig. 6e ) and strongly inhibited TNF-induced cleavage of PARP and caspase 3 ( Fig. 6f ). The ability of mPellino3 to rescue Pellino3-deficient MEFs from the enhanced apoptotic effects of TNF was lost when mutations (R131A/S161A) were introduced in its FHA domain, whereas mutations in its RING-like domain had no affect on the regulatory effects of mPellino3 on TNF signalling ( Fig. 6d–f ). These data again emphasize that loss of Pellino3 heavily biases the TNF pathway towards activation of the caspase cascade and ultimately apoptosis. The findings also highlight the important role for the FHA domain besides the dispensable nature of the RING-like domain in facilitating the ability of Pellino3 to counter-regulate the pro-apoptotic proclivity of TNF signalling. Given the important role of the FHA domain of Pellino3 in targeting RIP1 and regulating the pro-apoptotic effects of TNF, coupled to our earlier findings that the FHA domain of Pellino3 binds to RIP1 we also assessed if the FHA domain alone, of mPellino3, was sufficient to rescue Pellino3-deficient MEFs from the pro-apoptotic effects of TNF. However, reconstitution of Pellino3-deficient MEFs with mPellino3sΔC, which lacks the C-terminal RING-like domain but contains the FHA domain, was incapable of inhibiting the apoptotic effects of TNF/cycloheximide, based on the lack of effect on TNF-induced cell rounding/detachment ( Supplementary Fig. S7a ), annexin V staining ( Supplementary Fig. S7b ) and cleavage of PARP and caspase 3 ( Supplementary Fig. S7c ). This is consistent with our earlier findings demonstrating that the FHA domain of Pellino3 is not sufficient to inhibit TNF-induced recruitment of FADD and caspase 8 to RIP1 ( Fig. 5 ). Thus, while the FHA domain of Pellino3 is critically important in targeting RIP1 and manifesting the regulatory effects of Pellino3 on the TNF apoptotic pathway, the FHA domain alone is not sufficient to mediate the regulatory effects. This is consistent with a model in which the FHA domain mediates the binding of Pellino3 to RIP1 but there resides some additional anti-apoptotic function in Pellino3 that is lost with truncation of its C-terminal region. Given we hypothesize that Pellino3 regulates the pro-apoptotic effects of TNF by targeting RIP1, we further investigated the effect of Pellino3 deficiency in two models of TNF-induced apoptosis that show contrasting roles for RIP1. The first model involved cellular co-stimulation by TNF and Smac mimetics, that antagonize cIAPs by promoting their autoubiqutination and degradation, resulting in RIP1-dependent apoptosis [33] , [47] , [48] , whereas the second model involved co-stimulation with TNF and cycloheximide that induce apoptosis independently of the cell death role of RIP1 (refs 33 , 49 , 50 ). Intriguingly, the latter studies indicate that RIP1 has a pro-survival role under conditions of TNF/cycloheximide co-stimulation highlighting the differential roles of RIP1 under varying forms of TNF stimulation. We initially demonstrated that stimulation of wild-type bone marrow-derived macrophages (BMDMs) with TNF/Smac mimetic triggered apoptosis as indicated by increased Annexin V staining ( Fig. 7a ) and PARP/caspase 3 cleavage ( Fig. 7b ), and these pro-apoptotic markers were considerably enhanced in BMDMs from Pellino3 −/− mice. This was also confirmed in human cells by demonstrating that knockdown of Pellino3 expression in Hela cells augmented TNF/Smac mimetic-induced Annexin V staining ( Fig. 7c ) and PARP cleavage ( Fig. 7d ). Given the critical role for RIP1 in mediating TNF/Smac-induced apoptosis, these data are consistent with RIP1 being targeted by Pellino3 to regulate cell apoptosis. We next characterized TNF/cycloheximide-induced apoptosis in Pellino3-deficient cells. As we observed earlier, the apoptotic effects of TNF/cycloheximide, as indicated by Annexin V staining ( Fig. 7e ) and PARP cleavage ( Fig. 7f ), were greater in Pellino3 −/− than wild-type MEFs. We thus probed the role of RIP1 in mediating cell killing by TNF/cycloheximide. Knockdown of RIP1 expression in wild type and Pellino3-deficient MEFs strongly augmented TNF/cycloheximide-induced killing and this was inhibited by ZVAD ( Fig. 7e, f ), agreeing with previous reports that RIP1 has a pro-survival role in the TNF/cycloheximide model of apoptosis [33] , [49] , [50] . Interestingly, under conditions of RIP1 knockdown, TNF/cycloheximide induced similar levels of cell death in wild type and Pellino3 −/− , suggesting that RIP1 is required to manifest the regulatory effects of Pellino3 on TNF/cycloheximide-induced apoptosis. Intriguingly TNF/cycloheximide caused significant reduction in the levels of full-length RIP1 in Pellino3-deficient MEFs ( Fig. 7f , top panel) and this was coincident with the appearance of faster migrating forms of RIP1 (second panel Fig. 7f ). This was not observed in ZVAD-treated Pellino3 −/− cells, indicating that Pellino3 deficiency leads to increased caspase-mediated cleavage of RIP1 in response to TNF/cycloheximide, resulting in downregulation of the survival role of RIP1 and increased cell death. Given that caspase 8 has previously been reported to cleave RIP1 and promote TNF-induced apoptosis [34] , these data are consistent with our hypothesis in which Pellino3 targets RIP1 and prevents the interaction of RIP1 with caspase 8. Conversely, Pellino3 deficiency is associated with increased interaction of RIP1 and caspase 8, resulting in caspase 8-mediated cleavage of RIP1 and downregulation of its cell survival role in the TNF/cycloheximide model. 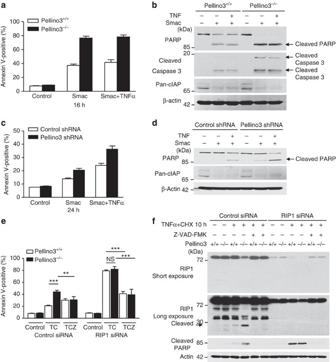Figure 7: Pellino3 deficiency sensitizes cells to TNF/Smac mimetic-induced apoptosis and TNF/cycloheximide-induced cleavage of RIP1. (a,b) Immortalized BMDMs from Pellino3+/+and Pellino3−/−mice were treated in the absence (control) or presence of murine TNF (40 ng ml−1) and/or Smac mimetic (10 μM) for 16 h. (c,d) Hela cells were infected with lentivirus containing constructs that encoded control or human Pellino3-specific shRNA. Cells were grown in the presence of puromycin to select for cells showing stable integration of shRNA constructs. Selected cells were treated in the absence (control) or presence of human TNF (40 ng ml−1) and/or Smac mimetic BV6 (10 μM) for 24 h. (a,c) Cells were analysed by flow cytometry for percentage of cells staining positive for annexin V. Data represent the mean +/− s.e.m. of two independent experiments. (b,d) Cell lysates were probed by immunoblotting using antibodies against PARP, cleaved caspase 3, pan-cIAP and β-actin. Cleaved forms of PARP and caspase 3 are indicated by arrows. (e,f) MEFs were isolated from Pellino3+/+and Pellino3−/−embryos and transfected with control or RIP1-specific siRNA. After 48 h, cells were treated in the absence (control) or presence of murine TNF (40 ng ml−1) plus cycloheximide (CHX) (10 μg ml−1) (TC) or murine TNF plus cycloheximide plus ZVAD (20 μM) (TCZ) for 10 h. (e) Cells were analysed by flow cytometry for percentage of cells staining positive for annexin V. Data represent the mean +/− s.e.m. of three independent experiments. **P<0.01; ***P<0.001 (two-way ANOVA). (f) Cell lysates were probed by immunoblotting for expression levels of RIP1, cleaved PARP and β-actin. The autoradiograph for the RIP1 immunblot was exposed for short and long times. Full-length images of immunoblots are shown inSupplementary Fig. S14. Figure 7: Pellino3 deficiency sensitizes cells to TNF/Smac mimetic-induced apoptosis and TNF/cycloheximide-induced cleavage of RIP1. ( a , b ) Immortalized BMDMs from Pellino3 +/+ and Pellino3 −/− mice were treated in the absence (control) or presence of murine TNF (40 ng ml −1 ) and/or Smac mimetic (10 μM) for 16 h. ( c , d ) Hela cells were infected with lentivirus containing constructs that encoded control or human Pellino3-specific shRNA. Cells were grown in the presence of puromycin to select for cells showing stable integration of shRNA constructs. Selected cells were treated in the absence (control) or presence of human TNF (40 ng ml −1 ) and/or Smac mimetic BV6 (10 μM) for 24 h. ( a , c ) Cells were analysed by flow cytometry for percentage of cells staining positive for annexin V. Data represent the mean +/− s.e.m. of two independent experiments. ( b , d ) Cell lysates were probed by immunoblotting using antibodies against PARP, cleaved caspase 3, pan-cIAP and β-actin. Cleaved forms of PARP and caspase 3 are indicated by arrows. ( e , f ) MEFs were isolated from Pellino3 +/+ and Pellino3 −/− embryos and transfected with control or RIP1-specific siRNA. After 48 h, cells were treated in the absence (control) or presence of murine TNF (40 ng ml −1 ) plus cycloheximide (CHX) (10 μg ml −1 ) (TC) or murine TNF plus cycloheximide plus ZVAD (20 μM) (TCZ) for 10 h. ( e ) Cells were analysed by flow cytometry for percentage of cells staining positive for annexin V. Data represent the mean +/− s.e.m. of three independent experiments. ** P <0.01; *** P <0.001 (two-way ANOVA). ( f ) Cell lysates were probed by immunoblotting for expression levels of RIP1, cleaved PARP and β-actin. The autoradiograph for the RIP1 immunblot was exposed for short and long times. Full-length images of immunoblots are shown in Supplementary Fig. S14 . Full size image In the above model, we observed increased TNF killing in Pellino3-deficient cells in the presence of the protein synthesis inhibitor cycloheximide and this suggested to us that the regulatory effects of Pellino3 on apoptosis are independent of NFκB and its induction of anti-apoptotic proteins. To further evaluate this possibility, we characterized the effect of Pellino3 deficiency on TNF-induced activation of NFκB and as expected the ability of TNF to activate the NFκB and MAPK pathways in Pellino3-deficient MEFs was intact ( Fig. 8a ). Indeed, the phosphorylation of IκBα in response to TNF stimulation was slightly more prolonged in Pellino3 −/− MEFs and this is consistent with modest augmentation of TNF-induced expression of the pro-inflammatory and NFκB-responsive gene IL-6 ( Fig. 8b ). Furthermore, the TNF-induced expression levels of the anti-apoptotic genes Bcl-x ( Fig. 8c ), A20 ( Fig. 8d ) and c-FLIP ( Fig. 8e ) were not reduced in Pellino3 −/− MEFs. These data strongly support our earlier contention that loss of Pellino3 increases the ability of TNF to induce apoptosis by a mechanism that involves increased interaction of RIP1 with caspase 8/FADD and is not dependent on inhibition of NF-κB. In order to directly confirm that the regulatory effect of Pellino3 on TNF-induced apoptosis is independent of the NFκB, a super repressor (SR) form of the inhibitory protein IκBα (IκBαSR) was overexpressed in wild type and Pellino3 −/− MEFs to block all TNF-induced activation of NFκB ( Fig. 9a ). Under these conditions of NFκB blockade, the pro-apoptotic effects of TNF were still augmented in Pellino3 −/− MEFs as evidenced by enhanced Annexin V staining ( Fig. 9b ) and PARP cleavage ( Fig. 9c ). These findings again support our hypothesis that Pellino3 targets TNF cell killing independently of the NFκB pathway. 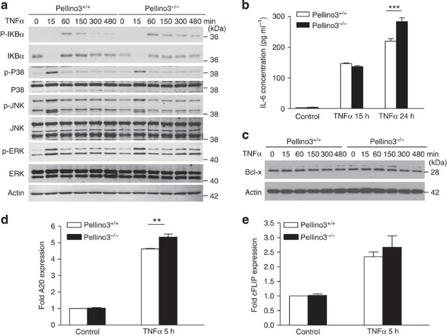Figure 8: TNF signalling in Pellino3−/−-deficient MEFs. MEFs were isolated from Pellino3+/+and Pellino3−/−embryos and treated in the absence (control) or presence of murine TNF (20 ng ml−1) for the indicated time periods. (a) Cell lysates were prepared and immunoblotted for expression levels of phosphorylated IκBα (p-IκBα), JNK (p-JNK), P38 (p-P38), ERK (p-ERK) and total levels of IκBα, JNK, P38 and ERK. Lysates were also probed for levels of β-actin to act as loading controls. (b) Conditioned media from treated cells were assayed for levels of IL-6 by ELISA. ***,P<0.001 (two-way ANOVA). (c) Cell lysates were probed by immunoblotting for expression levels of Bcl-x and β-actin. (d,e) mRNA expression levels of (d) A20 and (e) c-FLIP were measured by quantitative RT-PCR and expressed relative to expression levels in unstimulated Pellino3+/+MEFs. Data represent the mean +/− s.e.m. of three independent experiments; **P<0.01 (two-way ANOVA). Full-length images of immunoblots are shown inSupplementary Fig. S15. Figure 8: TNF signalling in Pellino3 −/− -deficient MEFs. MEFs were isolated from Pellino3 +/+ and Pellino3 −/− embryos and treated in the absence (control) or presence of murine TNF (20 ng ml −1 ) for the indicated time periods. ( a ) Cell lysates were prepared and immunoblotted for expression levels of phosphorylated IκBα (p-IκBα), JNK (p-JNK), P38 (p-P38), ERK (p-ERK) and total levels of IκBα, JNK, P38 and ERK. Lysates were also probed for levels of β-actin to act as loading controls. ( b ) Conditioned media from treated cells were assayed for levels of IL-6 by ELISA. ***, P <0.001 (two-way ANOVA). ( c ) Cell lysates were probed by immunoblotting for expression levels of Bcl-x and β-actin. ( d , e ) mRNA expression levels of ( d ) A20 and ( e ) c-FLIP were measured by quantitative RT-PCR and expressed relative to expression levels in unstimulated Pellino3 +/+ MEFs. Data represent the mean +/− s.e.m. of three independent experiments; ** P <0.01 (two-way ANOVA). Full-length images of immunoblots are shown in Supplementary Fig. S15 . 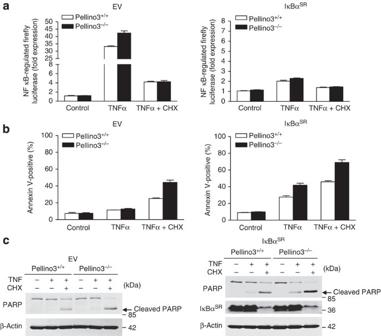Figure 9: The regulatory effect of Pellino3 on TNF-induced apoptosis is not mediated by NFκB. MEFs from Pellino3+/+and Pellino3−/−embryos were co-transfected with a NFκB-regulated firefly luciferase gene and an expression vector encoding a super repressor form of IκBα (IκBαSR) or an empty vector (EV). Cells were treated in the absence (Control) or presence of murine TNF (50 ng ml−1) and cycloheximide (CHX) (10 μg ml−1) for 8 h. (a) Data are presented as normalized luciferase expression relative to unstimulated cells. (b) Cells were analysed by flow cytometry for percentage of cells staining positive for annexin V. Data represent the mean +/− s.e.m. of two independent experiments. (c) Cell lysates were probed by immunoblotting for expression levels of PARP, IκBα and β-actin. A cleaved form of PARP is indicated by an arrow. Full-length images of immunoblots are shown inSupplementary Fig. S16. Full size image Figure 9: The regulatory effect of Pellino3 on TNF-induced apoptosis is not mediated by NFκB. MEFs from Pellino3 +/+ and Pellino3 −/− embryos were co-transfected with a NFκB-regulated firefly luciferase gene and an expression vector encoding a super repressor form of IκBα (IκBα SR ) or an empty vector (EV). Cells were treated in the absence (Control) or presence of murine TNF (50 ng ml −1 ) and cycloheximide (CHX) (10 μg ml −1 ) for 8 h. ( a ) Data are presented as normalized luciferase expression relative to unstimulated cells. ( b ) Cells were analysed by flow cytometry for percentage of cells staining positive for annexin V. Data represent the mean +/− s.e.m. of two independent experiments. ( c ) Cell lysates were probed by immunoblotting for expression levels of PARP, IκBα and β-actin. A cleaved form of PARP is indicated by an arrow. Full-length images of immunoblots are shown in Supplementary Fig. S16 . Full size image To further cement this hypothesis we directly measured complex II formation in response to TNF in Pellino3 −/− MEFs and also characterized TNF-induced formation of complex I, because the latter is a key signalling intermediate leading to downstream activation of NFκB. Wild type and Pellino3-deficient MEFs were thus stimulated with TNF for short times and immunoprecipitated TNFR1 was analysed for co-precipitation of complex I components. In wild-type MEFs, TNF promoted time-dependent recruitment of RIP1, TRAF2, TAK1 and NEMO to TNFR1 ( Fig. 10a ), a classical signature of complex I formation. The recruitment of these various components was unaffected in Pellino3 −/− MEFs thus excluding a role for Pellino3 in regulating TNF-induced formation of Complex I. Interestingly, the formation of Complex I is facilitated by the association of a number of these signalling proteins with ubiquitinated RIP1 and given that our earlier findings had indicated the targeting of RIP1 to be an important mechanism contributing to the regulatory effects of Pellino3 on apoptosis, we investigated the effect of Pellino3 deficiency on the ubiquitination status of RIP1. However, TNF induced the ubiquitination of RIP1 in both wild type and Pellino3-deficient cells with only very modest reduction in the latter cells ( Fig. 10b ). This is consistent with the lack of an important involvement for Pellino3 in regulating Complex I formation and in downstream activation of NFκB in response to TNF. We next characterized the effects of Pellino3 deficiency on TNF-induced formation of complex II. Wild type and Pellino3 −/− MEFs were stimulated with TNF for longer time periods and complex II was measured by immunoprecipitation of FADD and probing for the components RIP1 and caspase 8. In wild-type cells, TNF induced modest interaction of RIP1 and caspase 8 with FADD but these interactions were accelerated and strongly enhanced in Pellino3 −/− MEFs ( Fig. 10c ). Such enhanced formation of complex II was not restricted to MEFs from Pellino3-deficient mice because Pellino3 −/− BMDMs, relative to wild-type cells, showed greatly augmented interaction of caspase 8 and RIP1 with FADD, in response to TNF/Smac mimetic co-stimulation ( Fig. 10d ). Such increased complex II formation in Pellino3-deficient MEFs and BMDMs correlates closely with the more pronounced apoptotic features (described above) in response to TNF in these Pellino3 −/− cells. Again these findings are consistent with a model in which Pellino3 regulates the pro-apoptotic tendencies of TNF by targeting RIP1/caspase 8/FADD complex formation and not indirectly by affecting Complex I formation or NFκB activation. 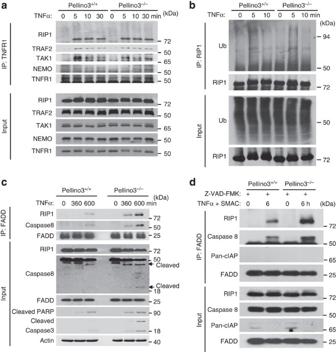Figure 10: Pellino3-deficient MEFs show enhanced levels of complex II but no effect on complex I formation in response to TNF. (a) MEFs were treated with TNF (40 ng ml−1) for the indicated times. Cell lysates were immunoprecipitated with an anti-TNFR1 antibody. Immunoprecipitates and cell lysates (‘input’) were probed for levels of RIP1, TRAF2, TAK1, NEMO and TNFR1 by immunoblotting. (b) MEFs were treated with TNF (40 ng ml−1) for the indicated times and followed by immunoprecipitation of endogenous RIP1. Immunoprecipitates and cell lysates (‘input’) were probed using anti-ubiquitin and -RIP1 antibodies. (c) MEFs were isolated from Pellino3+/+and Pellino3−/−embryos and treated with TNF (1.5 μg ml−1) for the indicated times. Complex II was immunoprecipitated using an anti-FADD and analysed for co-precipitated RIP1 and caspase 8. The whole-cell lysates (input) were immunoblotted using RIP1, caspase 8, FADD, cleaved PARP, cleaved caspase 3 and β-actin antibodies. Cleaved forms of caspase 8 are indicated by arrows (d) Immortalized BMDMs from Pellino3+/+and Pellino3−/−mice were treated in the absence (control) or presence of murine TNF (40 ng ml−1) and Smac mimetic (10 μM) for 16 h. Cells were also treated with ZVAD to prevent activation of caspase 8 and cell death. Cell lysates were immunoprecipitated using an anti-FADD antibody and analysed for co-precipitated RIP1 and caspase 8. The whole-cell lysates (input) were immunoblotted using RIP1, caspase 8, pan-cIAP and FADD antibodies. Full-length images of immunoblots are shown inSupplementary Fig. S17. Figure 10: Pellino3-deficient MEFs show enhanced levels of complex II but no effect on complex I formation in response to TNF. ( a ) MEFs were treated with TNF (40 ng ml −1 ) for the indicated times. Cell lysates were immunoprecipitated with an anti-TNFR1 antibody. Immunoprecipitates and cell lysates (‘input’) were probed for levels of RIP1, TRAF2, TAK1, NEMO and TNFR1 by immunoblotting. ( b ) MEFs were treated with TNF (40 ng ml −1 ) for the indicated times and followed by immunoprecipitation of endogenous RIP1. Immunoprecipitates and cell lysates (‘input’) were probed using anti-ubiquitin and -RIP1 antibodies. ( c ) MEFs were isolated from Pellino3 +/+ and Pellino3 −/− embryos and treated with TNF (1.5 μg ml −1 ) for the indicated times. Complex II was immunoprecipitated using an anti-FADD and analysed for co-precipitated RIP1 and caspase 8. The whole-cell lysates (input) were immunoblotted using RIP1, caspase 8, FADD, cleaved PARP, cleaved caspase 3 and β-actin antibodies. Cleaved forms of caspase 8 are indicated by arrows ( d ) Immortalized BMDMs from Pellino3 +/+ and Pellino3 −/− mice were treated in the absence (control) or presence of murine TNF (40 ng ml −1 ) and Smac mimetic (10 μM) for 16 h. Cells were also treated with ZVAD to prevent activation of caspase 8 and cell death. Cell lysates were immunoprecipitated using an anti-FADD antibody and analysed for co-precipitated RIP1 and caspase 8. The whole-cell lysates (input) were immunoblotted using RIP1, caspase 8, pan-cIAP and FADD antibodies. Full-length images of immunoblots are shown in Supplementary Fig. S17 . Full size image Exacerbation of TNF toxicity in Pellino3-deficient mice The findings above provide strong evidence for a role for Pellino3 in regulating apoptosis in response to TNF. We next investigated the in vivo relevance of this role using Pellino3-deficient mice. In order to define the in vivo role of Pellino3 in the context of the toxic effects of TNF the well-established liver injury model was employed in which the hepatotoxic agent D -galactosamine ( D -gal) sensitizes mice to the lethal effects of low doses of TNF. We co-administered D -gal with sub-optimal levels of TNF that failed to render Pellino3 +/+ mice sensitive to the lethal effects of TNF ( Fig. 11a ). However, under these same conditions TNF caused lethality in all Pellino3 −/− mice 24 h after administration of TNF. The administration of D -gal alone had no affect on the survival of Pellino3 +/+ or Pellino3 −/− mice. Given that hepatoxicity is the key contributing factor to the lethal effects in this model, liver tissue was examined from the different mouse cohorts. We observed multifocal areas of haemorrhage in Pellino3 −/− mice that had been co-administered with D -gal and TNF, whereas no such effects were apparent in Pellino3-deficient mice that had not been challenged with TNF or in wild-type control mice irrespective of the administration regime ( Fig. 11b ). No significant microscopic abnormalities were detected on examination of hepatic tissue from D -gal-treated wild-type and Pellino3-deficient mice ( Fig. 11c , left panels). Co-administration of D -gal and TNF to Pellino3 +/+ mice lead to widespread swelling of hepatocytes due to microvesicular vacuolation and fine granulation of the cytoplasm leading to compression of sinus structures. This is typical of an adaptive cell response to injury coupled with proliferation of hepatic drug-metabolizing enzymes as a result of D-gal treatment. In contrast, the same co-administration protocol in Pellino3 −/− mice led to widespread hepatocyte death with marked disruption of hepatocyte cord structures and part replacement by red blood cells. Individual hepatocytes were swollen with many cells containing karyorrhectic (fragmented) nuclei. The hepatocyte death observed in the latter group was apoptotic in nature because immunhistochemical analysis of the hepatic tissue clearly showed intense immunoreactivity with an anti-cleaved caspase 3 antibody ( Fig. 11c , right panels). This was further confirmed by western blot analysis demonstrating very high levels of cleaved caspase 3 and caspase 8 in hepatic tissue from Pellino3 −/− mice that had been challenged with D-gal and TNF ( Fig. 11d ). These data provide very strong evidence for a critical physiological role for Pellino3 in regulating the potential toxic effects of TNF. Furthermore, the severe hepatotoxicity observed in the Pellino3 −/− mice reflects a role for Pellino3 in directly regulating the apoptotic process rather than modulating a systemic inflammatory response, because lack of Pellino3 fails to affect circulating serum levels of IL-6, IL-10 or TNF ( Fig. 11e ). In conjunction with the earlier cell-based approaches these in vivo findings provide strong support for Pellino3 acting as a novel factor in TNF biology. The high sensitivity of Pellino3 −/− mice to the lethal effects of TNF strongly promotes Pellino3 as a crucial factor in determining whether cells survive or die in response to TNF challenge. 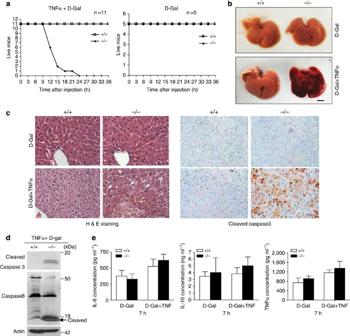Figure 11: Loss of Pellino3 in mice leads to increased hepatoxicity and lethality in response to TNFin vivo. Age- and sex-matched Pellino3+/+and Pellino3−/−mice were injected intraperitoneally with TNF and D-galactosamine (n=11) or D-galactosamine alone (n=5). (a) Survival was monitored every hour for 36 h. (b) Liver tissues were collected and photographed at 12 h after injection. Scale bar, 3 mm. (c) Hepatic tissue was collected 12 h after injection, sectioned and subjected to histological analysis using H&E staining and immunohistochemistry using anti-cleaved caspase 3 antibody. The white arrows indicate hepatocytes with fragmented nuclei. Scale bar, 50 μm. (d) Cell lysates were generated from hepatic tissue 12 h post injection and probed by immunoblotting for levels of cleaved caspase 3, caspase 8 and β-actin. (e) Blood samples were taken from mice 7 h after injection and serum assayed by ELISA for levels of IL-6, IL-10 and TNF. Data represent the mean +/− s.e.m. of four independent experiments. Full-length images of immunoblots are shown inSupplementary Fig. S18. Figure 11: Loss of Pellino3 in mice leads to increased hepatoxicity and lethality in response to TNF in vivo . Age- and sex-matched Pellino3 +/+ and Pellino3 −/− mice were injected intraperitoneally with TNF and D-galactosamine ( n =11) or D-galactosamine alone ( n =5). ( a ) Survival was monitored every hour for 36 h. ( b ) Liver tissues were collected and photographed at 12 h after injection. Scale bar, 3 mm. ( c ) Hepatic tissue was collected 12 h after injection, sectioned and subjected to histological analysis using H&E staining and immunohistochemistry using anti-cleaved caspase 3 antibody. The white arrows indicate hepatocytes with fragmented nuclei. Scale bar, 50 μm. ( d ) Cell lysates were generated from hepatic tissue 12 h post injection and probed by immunoblotting for levels of cleaved caspase 3, caspase 8 and β-actin. ( e ) Blood samples were taken from mice 7 h after injection and serum assayed by ELISA for levels of IL-6, IL-10 and TNF. Data represent the mean +/− s.e.m. of four independent experiments. Full-length images of immunoblots are shown in Supplementary Fig. S18 . Full size image This study highlights a critical role for Pellino3 in regulating the pro-apoptotic effects of TNF. The initial suggestion of such a role arose from our human cell line studies in which Pellino3 knockdown augmented the apoptotic effects of TNF. This regulatory role for Pellino3 was observed in a number of cell types indicating an important function for Pellino3 in various TNF-responsive cells. The physiological relevance of Pellino3 in the TNF pathway was confirmed by the generation of Pellino3-deficient mice with cells from these mice displaying increased sensitivity to the pro-apoptotic effects of TNF. Furthermore Pellino3-deficient mice showed greatly increased susceptibility to the lethal effects of TNF and this was associated with increased severity of TNF-induced hepatotoxicity. All of these findings strongly promote Pellino3 as a regulator of the apoptotic pathway that is triggered by TNF and provides the first data showing that a member of the Pellino family can regulate TNF signalling. Given that NF-κB acts to counter-regulate the apoptotic pathway by the induction of anti-apoptotic proteins, it was of interest to examine whether Pellino3 could exert its regulatory effects on TNF-induced apoptosis by affecting the NF-κB pathway. However, the increased apoptosis that is observed in Pellino3 knockdown or -deficient cells cannot be easily explained by the regulation of NF-κB, because we observed increased TNF killing in Pellino3-deficient cells in the presence of the protein synthesis inhibitor cycloheximide, and the augmented pro-apoptotic effects of TNF, under conditions of Pellino3 deficiency, are still observed when the NFκB pathway is blocked by IκBαSR. Furthermore, cells lacking Pellino3 do not show any deficit in the activation of the NF-κB in response to TNF. Indeed, there appears to be a modest augmentation of the NF-κB pathway in such cells in response to TNF, suggesting that Pellino3 may exert some negative influence on NF-κB. This is consistent with a previous report indicating that Pellino3 may negatively regulate IL-1-induced activation of NF-κB [51] . Furthermore, Peli1 has been recently shown to inhibit T cell activation by downregulating the NF-κB subunit c-Rel [52] , indicating that the Pellino family may serve important roles in controlling the activation of NF-κB. Given that the targeting of the NF-κB pathway by Pellino3 does not provide an underlying basis to its regulatory effects on apoptosis, we probed a direct role for Pellino3 in the apoptotic pathway. Our findings demonstrate that Pellino3 has an important role in controlling complex II formation in response to TNF. We show that Pellino3 can interact with the complex II components, caspase 8 and RIP1, with the latter interaction being driven by TNF. Indeed, the targeting of RIP1 by Pellino3 appears to be important in mediating the regulatory effects of Pellino3 on TNF-induced apoptosis because mutants of Pellino3 that lack the ability to interact with RIP1, while still associating with caspase 8, fail to regulate complex II formation or progression to apoptosis in response to TNF. It is especially intriguing that the targeting of RIP1 by Pellino3 is a key part of the regulatory process given the pivotal role of RIP1 in determining cell fate in response to TNF challenge. The ubiquitination of RIP1 by E3 ligases, such as the IAPs, has traditionally been associated with promoting formation of Complex I and activation of the NF-κB pathway and blocking complex II formation by inhibiting the binding of RIP1 to FADD and caspase 8 (ref. 16 ). We thus considered the possibility that the negative regulatory effects of Pellino3 on complex II formation may be explained by Pellino3-induced ubiquitination of RIP1. However, in Pellino3-deficient cells we were unable to detect any major reduction in the ubiquitination of RIP1 in response to TNF and this is consistent with the lack of effect of Pellino3 deficiency on TNF-induced formation of Complex I and activation of NFκB. Furthermore, we show that the regulatory effects of Pellino3 on complex II formation and apoptosis are independent of its RING-like domain. This suggests that Pellino3 contains important regulatory functions independent of its E3 catalytic activity. Instead, the FHA domain of Pellino3 is crucially important in facilitating its regulatory effects on the pro-apoptotic effects of TNF. To date, the FHA domain of the Pellino family has been associated with mediating binding to the IRAK family members [40] but the present data identifies RIP1 as a key target for Pellino3, with the FHA domain of the latter being a key requirement for associating with RIP1. While the FHA domain has a critical role in mediating the regulatory effects of Pellino3, the C-terminal region of the protein is also required to manifest regulatory activity and this may reflect a need for Pellino3 to interact with caspase 8 because the FHA domain of Pellino3, which lacks the C-terminal region of the full-length protein, is unable to bind to caspase 8. Indeed, it will be interesting for future studies to explore the potential of Pellino3 to inhibit the activity of caspase 8 and/or access of the latter to its substrates, as this may also contribute to the regulatory effects of Pellino3 on TNF-induced apoptosis. The FHA domain is a phosphothreonine-binding module and the identification of potential recognition sites on RIP1 for the FHA domain of Pellino3 will add greatly to our understanding of this pathway. Indeed, it is interesting to note that while Pellino3 can interact directly with RIP1 in an in vitro setting, this is barely detectable and strong binding of RIP1 to Pellino3 is only manifested in a cell setting and in response to TNF stimulation. Thus TNF may induce the phosphorylation of RIP1 allowing for high-affinity recognition of RIP1 by the FHA domain of Pellino3. Indeed, our findings are consistent with a model where stimulation of cells with TNF promotes binding of Pellino3, via its FHA domain, to RIP1 and this inhibits the binding of FADD to RIP1. This will lead to reduced interaction of RIP1 and caspase 8 and so reduces the likelihood of triggering the apoptotic pathway. In a situation where Pellino3 is absent, this braking mechanism no longer applies, leading to increased complex II formation and apoptosis in response to TNF, even under circumstances where NF-κB activation has not been compromised. Our hypothesis that Pellino3 targets RIP1 as part of mediating its regulatory effects in the TNF pathway also serves to explain the apparent contrasting roles of RIP1 in TNF/Smac- and TNF/cycloheximide-induced apoptosis. The Smac mimetic mimics the activity of the mitochondrial protein Smac/Diablo by inhibiting IAP proteins and promoting autoubiquitination and degradation of cIAP1 and cIAP2, leading to loss of RIP1 ubiquitination and formation of complex II and RIP1-mediated downstream triggering of apoptosis [47] , [48] , [53] , [54] , [55] , [56] , [57] . In the TNF/Smac mimetic model, we show that Pellino3 negatively regulates the recruitment of RIP1 to Complex II and so represses the pro-death role of RIP1 in this model. In contrast, we confirm previous reports that cell killing by TNF/cycloheximide is not mediated by RIP1 and instead RIP1 has a survival role under these conditions [33] , [49] , [50] . In this TNF/cycloheximide model, Pellino3 positively regulates the pro-survival role of RIP1 by limiting interaction of the latter with caspase 8 and so preventing caspase 8-induced cleavage of RIP1 and facilitating RIP1-mediated cell survival. The mechanism underlying such a survival role of RIP1 is not understood but studies to investigate the potential of RIP1 to decrease caspase activity in Complex II under these conditions may be informative. Furthermore, as Pellino3 also interacts with caspase 8 it is interesting to speculate that Pellino3 may work in conjunction with RIP1 to regulate the activity of caspase 8. We were also keen to explore if the regulatory effects of Pellino3 on the formation of a complex containing FADD, RIP1 and caspase 8 extended beyond pathways that are triggered by TNFR1. Intriguingly the effects of Pellino3 appear to show a high degree of specificity towards the TNF pathway, as we show that the pro-apoptotic effects of the related Fas pathway are not subject to regulation by Pellino3. Furthermore, two recent reports have characterized a death-inducing cytosolic complex containing FADD, RIP1 and caspase 8 that forms independently of death receptor activation but in response to intracellular stress [58] , [59] . These latter studies describe the formation of a complex termed the ‘Ripoptosome’ that contains FADD, RIP1 and caspase 8 and forms spontaneously in response to the depletion of cIAPs by IAP antagonists or the genotoxic compound etoposide. We explored the potential of Pellino3 to regulate the cell death pathways induced by etoposide, in MEFs, but like the Fas pathway, Pellino3 was without effect. However, our data does not fully exclude a potential role for Pellino3 in regulating etoposide-induced cell death in other cell types, especially cancer cells, given that etoposide has been shown to promote the interaction of RIP1 with caspase 8 in tumour but not normal cells [48] . Furthermore, while the mechanistic basis to the specificity of Pellino3 for the TNF pathway is unknown it may reside in Pellino3 targeting a unique component of the TNF signal transduction system or alternatively TNF may be unique in regulating or modifying Pellino3 to a state in which it can manifest its regulatory potential. The targeting of RIP1 by Pellino3 is of interest to Pellino biology given that Peli 1 has also been demonstrated to target RIP1 (ref. 37 ). However, the outcomes of such interactions differ at the functional and molecular levels. First, while Pellino3 targets RIP1 to regulate cell killing, Pellino1 interacts with RIP1 to promote activation of NF-κB, at least in the context of TLR3 and TLR4 signalling [37] . Second, while the interaction of Pellino3 with RIP1 and its regulatory effects on apoptosis are independent of its RING-like domain, Pellino1 is proposed to facilitate activation of the NF-κB pathway by catalysing polyubiquitination of RIP1 (ref. 37 ). Such varying roles for these members of the Pellino family is not without precedent because Pellino3 negatively regulates IL-1-induced activation of NFκB [51] , whereas Pellino1 acts as a positive regulator of IL-1 signalling [44] , although the latter suggestion has recently been challenged with findings from Pellino1-deficient mice [37] . It will be of great interest to explore the potential interplay between Pellino1 and Pellino3 in terms of regulating RIP function in the TNF pathway. While cell line studies suggest that Pellino1 is not involved in TNF signalling [44] the recent generation of Pellino1 knockout mice will allow for examination of its role in a more physiological setting. In summary the present findings highlight Pellino3 as a new factor in the TNF signalling pathway and indicate that it may have an important role in determining whether a cell survives or dies in response to TNF. The present study also adds to a growing appreciation of the diverse functions of the Pellino family in immune signalling pathways. While most studies to date have focused on Pellino proteins as regulators of IL-1 and TLR signalling, the present report extends their roles beyond these pathways. Furthermore, Peli1 has been described as an important regulator of T-cell activation and self tolerance [52] , [60] . Such findings, in conjunction with the present report, add to an increasing appreciation of the importance of the Pellino family in a variety of signalling pathways in the innate and adaptive immune systems. Pellino3-deficient mice Pellino3-deficient mice were generated by Taconic Artemis using its proprietary technology as previously described [46] . Briefly, a targeting vector, in which exon 3 of the Pellino3 gene was flanked by loxP sites, was designed to generate homologous recombinant ES clones that were used to generate chimeric mice. To make constitutive Pellino3 −/− mice, mice that were heterozygous for the targeted allele were bred with mice containing Cre recombinase regulated by the ROSA26 locus (C57BL/6 Gt(ROSA)26Sortm16(Cre)Arte). This results in the deletion of exon 3 and loss of function of the Pellino3 gene by generating a frameshift in all downstream exons. The Cre transgene was subsequently removed by breeding the Pellino3 +/− mice with C57BL/6 mice during colony expansion. Animal breeding and maintenance were performed in the Bioresource facility of National University of Ireland (NUI) Maynooth. All animal experiments were performed in accordance with protocols approved by the Research Ethics committee of NUI Maynooth. Eight-week-old male mice were used for in vivo studies. Cell culture Hela, HEK293 and 1321N1 cells were cultured in Dulbecco’s modified Eagle’s medium supplemented with 10% ( v / v ) fetal bovine serum (FBS), 100 μg ml −1 penicillin G and 100 μg ml −1 streptomycin. Cells were maintained at 37 °C in a humidified atmosphere of 5% CO 2 . For the preparation of primary MEFs, Pellino3 +/− mice were bred to generate Pellino3 +/+ and Pellino3 −/− embryos. Embryos were dissected from pregnant females at day 13 post coitum. MEFs were isolated by standard procedure and cultured in DMEM supplemented with 10% ( v / v ) FBS. Immortalized WT and Peli3 −/− BMDMs were kindly prepared by Dr Kate Fitzgerald (The University of Massachusetts Medical School, Worcester, Massachusetts, USA) and cultured in Dulbecco’s modified Eagle’s medium supplemented with 10% ( v / v ) FBS, 100 μg ml −1 penicillin G and 100 μg ml −1 streptomycin. Expression vectors The plasmids pcDNA3.1-Pellino3s-/3l-myc, Pellino3s(R131A/S161A)-myc (Pellino3sFHAm), Pellino3l(R155A/S185A)-myc (Pellino3lFHAm), Pellino3s(C360A/C363A)-myc (Pellino3sE3m) and Pellino3l (C384A/C387A)-myc (Pellino3lE3m), flag-Pellino3sΔC(1-313aa) and HA-caspase 8 (C360/A) were generated in-house. Pellino3s-flag was from Xiaoxia Li (Cleveland Clinic). Myc-RIP1 was from Xin Lin (University of Texas, M.D. Anderson Cancer Center). HA-RIP1 and CrmA were from JinWoo Kim (Korea Advanced Institute of Science and Technology). Caspase 8 (C360/A)-myc and flag-FADD were from A. Thorburn (University of Colorado at Denver and Health Sciences Center). IκBα SR was from Dr Martina Schröder (National University of Ireland, Maynooth, Ireland). Truncation mutants encoding the DED (1-194aa) and caspase (195–479aa) domains of caspase 8 were cloned into pcDNA4.0 vector. Myc-tagged Pellino3s, Pellino3l, Pellino3sFHAm and Pellino3lFHAm were subcloned into His-tagged pRSET-A (Invitrogen). Procaspase 8 and the caspase domain (195–479aa) of caspase 8 were cloned into the His-tagged vector pET-30a (Novagen). MPellino3 was cloned from embryo brain and into the retroviral MSCV2.2-IRES-GFP vector. FHA (R131A/S161A) (mP3Fm), RING-like domain (C360A/C363A) (mP3Em) and ΔC(1–313aa) mutants of mPellino were generated in house. Antibodies and reagents Anti-RIP1 (610459 BD) (1:1,000 working dilution) was from BD Transduction Labs; anti-caspase 8 (C-20; sc-6136) (for immunoprecipitations) (1:1,000), anti-IκBα (C-21; sc-371) (1:1,000), anti-TRAF2 (C-20; sc-876) (1:500), anti-TNFR1 (H-5; sc-8436) (1:500), anti-Tak1 (M-579; sc-7162) (1:500), anti-NEMO (FL-419; sc-8330) (1:500) and anti-Ub (P4D1; sc-8017) (1:500) were from Santa Cruz; anti-HA (2367) (1:1,000), anti-Myc (2276) (1:2,000), anti-PARP (9542) (1:2,000), anti-cleaved caspase 3 (9664) (1:500), anti-caspase 8 (9746) (1:500), anti-p-IκBα (9246) (1:500), anti-JNK(9252) (1:1,000), anti-P38 (9212) (1:1,000), anti-Erk (9102) (1:2,000), anti-p-JNK (9251) (1:1,000), anti-p-ERK (9101) (1:1,000), and anti-p-P38 (9211) (1:1,000) were from Cell Signaling; anti-caspase 8 (mouse) (1G12; ALX-804-447) (1:1,000) and anti-FADD (1F7; AAM-212) (1:1,000) were from Enzo Life Science; anti-human and mouse TNFR1 (AF225; AF-425-PB) (for immunoprecipitations) (1:1,000) and anti-human and mouse Pan-cIAP (MAB3400) (1:1,000) were from R&D Systems; anti-β-actin (AC-15; A 1978) (1:10,000) was from Sigma; anti-Pellino3 antibodies (1:1,000) were generated in-house; anti-mouse IRDyeTM 700 (1:5,000), anti-rabbit IRDyeTM 800 (1:5,000) and anti-rabbit IRDyeTM 700 light chain (1:5,000) were from LI-COR Biosciences; anti-goat IRDyeCW800 (1:10,000) was from Rockland; anti-mouse-HRP (1:5,000) was from Cell Signaling; anti-rabbit-HRP (1:5,000) was from Promega; anti-Goat-HRP (1:5,000) was from Santa Cruz; TNFα was from R&D Systems; anti-Fas (554255) was from BD Pharmingen; Etoposide (E1383) and Cycloheximide (C4859) were from Sigma; ZVAD-FMK (G7232) was from Promega. SMAC peptide was a gift from Professor Luke O'Neill (Trinity College Dublin, Ireland). BV6 was a gift from Professor Harald Wajant (University Hospital Würzburg, Germany). Preparation and transfection of siRNA Human Pellino3-specific siRNA (sense: 5′-GCACAGCAUCUCGUAUACATT-3′; antisense: 5′-UGUAUACGAGAUGCUGUGCTG3-3′) and murine RIP1-specific siRNA (sense: 5′-GGUGGUACCCUUUACUACATT-3′; antisense: 5′-UGUAGUAAAGGGUACCACCAT-3′) were from Ambion. Cells were transfected by Lipofectamine 2000 according to the manufacturer’s instructions and allowed to recover for 48 h prior to experiments. Pellino3 knockdown by lentiviral shRNA in human cells Lentiviral constructs encoding human Pellino3 shRNA were purchased from Sigma. The shRNA sequence specifically targeted the 3′ UTR of Pellino3 and had the following sequence: GCACTTGCTGATAGCCACTATCCGGGCACTTGCTGATAGCCACTATCTCGAGATAGTGGC TATCAGCAAGTGCTTTTTTG. Constructs were co-transfected with packaging and envelope plasmids (dR89.1 and VSV-G) into 293T cells, and lentivirus from the medium supernatants was used to infect Hela, HEK293 and 1321N1 cells. Cells were subsequently grown for 1 week under puromycin (10 μg ml −1 ) selection. The knockdown efficiency was assessed by the immunoblotting of whole-cell lysates. Control cells were infected with lentivirus containing a nontargeting shRNA vector that encodes for shRNA that does not match any known human or mouse gene. For rescue assays, expression constructs encoding myc-tagged wild type or mutated forms of Pellino3 were transfected into puromycin-selected cells. Cells were then assessed for various features associated with apoptosis. Real-time PCR assays Real-time PCR analyses were performed using TaqMan Gene Expression kits (Finnzymes), according to the manufacturer’s instructions. The following primers were used to amplify the fragments of the indicated genes: mA20, forward, 5′-TGCCAGTTTTGCCCACAGT-3′ and reverse, 5′-TTCAGAGCCACGAGCTTCCT-3′; mcFlip, forward, 5′-GCTCCAGAATGGGCGAAGT-3′ and reverse, 5′-CACGGATGTGCGGAGGTAA-3′. Each mRNA quantification was normalized relative to the housekeeping gene hypoxanthine phosphoribosyltransferase 1 (HPRT) using the primers; mHPRT forward, 5′-GTCCCAGCGTCGTGATTAGC-3′ and reverse, 5′-TGGCCTCCCATCTCCTTCA-3′. Immunoprecipitation and western blot analysis Cells were grown in six-well plates and then transfected with designated expression constructs. For TNFR1-associated complex I analysis, cells were stimulated for various times with TNFα (50 ng ml −1 ). For DISC complex II analysis, cells were stimulated for various times with TNFα (40 ng ml −1 ), cycloheximide (10 μg ml −1 ) and ZVAD-FMK (20 μm). Cells were subsequently harvested in 500 μl of lysis buffer (20 mM Tris–HCl (pH 7.4), containing 150 mM NaCl, 0.2% ( v / v ) Igepal, 10% ( w / v ) Glycerol, 50 mM NaF, 1 mM Na 3 VO 4 , 1 mM phenylmethylsulfonyl fluoride and complete protease inhibitor cocktail (Roche)) and incubated at 4 °C for 30 min with gentle rocking. Cell lysates were centrifuged at 14,000 g for 10 min to remove cell debris and nuclei. An aliquot (50 μl) of the supernatant was retained for western blot analysis, and the remainder was subjected to immunoprecipitation. Cell lysates were initially precleared by incubating with non immune IgG antibody (1 μg) and protein A/G agarose (10 μl) for 1 h at 4 °C with rocking followed by rapid centrifugation of the agarose beads. Each supernatant was removed to a fresh microcentrifuge tube followed by addition of the appropriate antibody (2 μg) and incubated for 24 h at 4 °C with rocking. An aliquot (50 μl) of protein A/G agarose was added to each sample and incubated with rocking overnight at 4 °C. Immunoprecipitates were collected by passing the samples through Cytosignal filters by centrifugation at 16,000 g for 1 min at 4 °C. The trapped beads were then washed four times with 500 μl of lysis buffer (without Na 3 VO 4 , dithiothreitol, phenylmethylsulfonyl fluoride or protease inhibitor cocktail). An aliquot (60 μl) of SDS–PAGE sample buffer was added to the trapped beads and the immunoprecipitated proteins were eluted by centrifugation at 16,000 g for 1 min. Samples were boiled for 5 min, resolved by SDS–PAGE, transferred to nitrocellulose membranes and analysed by immunoblotting using the appropriate antibodies. Immunoreactivity was visualized by the Odyssey Imaging System (LI-COR Biosciences) or enhanced chemiluminescence. Generation of recombinant proteins and in vitro binding assays Myc-tagged Pellino3s, Pellino3l, Pellino3sFHAm and Pellino3lFHAm were cloned into the His-tagged vector pRSET-A (Invitrogen). Procaspase 8, the caspase domain (195–479aa) of caspase 8 and RIP1 were cloned into the His-tagged vector pET-30a (Novagen). The constructs were transformed into Escherichia coli cells, protein expression induced by IPTG and recombinant proteins purified from cell lysates by affinity chromatography using nickel–nitrilotriacetic acid–agarose (Qiagen) according to the manufacturer’s instructions. The purity and integrity of recombinant proteins were confirmed by subjecting samples to SDS–PAGE (followed by Coomassie staining) in addition to western blotting using the appropriate antibodies. For the in vitro binding assays characterizing the binding of Pellino3 to partner proteins, recombinant myc-tagged Pellino3 proteins (1 μg) were initially immunoprecipitated in binding buffer (20 mM Tris–HCl (pH 7.4), containing 150 mM NaCl, 0.2% ( v / v ) Igepal, 10% ( w / v ) glycerol and complete protease inhibitor cocktail) using an anti-myc antibody (2 μg) and protein A/G beads (30 μl) as above. The beads were washed five times with binding buffer and then incubated overnight at 4 °C with purified recombinant forms of procaspase 8 or its caspase domain (300 ng) or recombinant RIP1(200 ng) or lysates (300 μl per well of six-well plates) from HEK293 cells previously transfected with HA-tagged RIP1. Beads were subjected to serial washes with binding buffer followed by centrifugation. Co-precipitated proteins were eluted in SDS–PAGE sample buffer and then subjected to western blot analysis. In Vitro K63 ubiquitination assay Recombinant Pellino3s, P3sFHAm or P3sE3m protein (0.5 μg) were incubated with ubiquitin (with all lysine residues, except residue 63, mutated to arginine (K63 only) (2 μg), E1 (50 ng), UbcH13 (400 ng) and protease inhibitor mixture (EDTA-free) in 5 mM Tris-HCl (pH 7.5) containing 2 mM MgCl 2 , 2 mM ATP and 100 mM NaCl. Reactions were incubated at 37 °C for 2 h and terminated by the addition of SDS–PAGE sample buffer. Samples were boiled for 5 min, resolved by SDS–PAGE, transferred to nitrocellulose membranes and analysed by immunoblotting using an anti-ubiquitin antibody. FACS Wild type and Pellino3 knockdown or knockout cells were treated as indicated and assayed for programmed cell death using an Annexin V-FITC Apoptosis Detection Kit (BD Pharmingen) according to the manufacturer’s instructions. Briefly, cells were washed once in PBS and then in binding buffer (10 mM Hepes (pH 7.4), containing 140 mM NaCl and 2.5 mM CaCl 2 ). Washed cells were resuspended in binding buffer (1–5 × 10 6 cells per ml) and aliquots (100 μl) of resuspended cells were incubated for 15 min at room temperature in the dark with Annexin V-FITC (5 μl). Binding buffer (400 μl) was added to each sample followed by flow cytometric analysis of Annexin V-reactive cells using a FACSCalibur flow cytometer and CellQuest software (BD Biosciences). MTT assays Control and Pellino3 knockdown cells were grown in 48-well plates and then stimulated with TNFα (40 ng ml −1 ) and cycloheximide (10 μg ml −1 ) or cycloheximide alone for indicated times. 3-(4, 5-dimethylthiazol-2-yl)-2, 5-diphenyltetrazolium bromide (MTT) (5 mg ml −1 ) was added to the cells and incubated for 3 h at 37 °C. Media was removed and DMSO added to solubilize the cells. The absorbance of the solubilized material was measured at 540 nm using a BioTEK Microplate Reader and this was used as an index of mitochondrial activity and thus cell viability. Retroviral rescue assay MSCV plasmid or MSCV-mPellino3 (mP3), MSCV-mP3Fm and MSCV-mP3Em or MSCV-mP3ΔC (1 μg) were co-transfected with the packaging vector ψ (1 μg) into 293T cells. After 48 h, the retrovirus-containing medium was harvested and used to infect Pellino3-deficient MEFs in 25-cm 2 flasks. The flasks were incubated at 37 °C for 48 h prior to experiments. In vivo toxicity studies involving TNF and D -galactosamine Age- and sex-matched wild-type and Pellino3-deficient mice were injected intraperitoneally with TNF (0.0025 μg g −1 body weight) plus D -galactosamine (0.8 mg g −1 body weight). Mouse survival was monitored over a time period of 36 h. In some experiments mice were killed 12 h after injection, liver samples collected and processed for immunohistochemical analysis. In other cases serum samples were obtained 7 h after injection and assayed for levels of IL-6, IL-10 and TNF using sandwich ELISA kits according to the manufacturer’s instructions (R&D Systems). Immunohistochemical analysis At post-mortem examination samples of liver tissue were fixed in neutral buffered formalin. Following fixation tissues were paraffin-embedded, sectioned at 5 μm and stained with haematoxylin and eosin (H&E). For detection of cleaved caspase 3, sections were initially deparaffinized and incubated in 0.3% ( v / v ) H 2 O 2 (Fluka) for 30 min for blockade of endogenous peroxidase activity. Sections were blocked with PBS containing 5% ( v / v ) goat serum (Vector) and then incubated with anti-cleaved caspase 3 antibody (9664; Cell Signalling). The Vectastain ABC kit (PK-6100; Vector Laboratories) was used according to the manufacturer’s specifications for detection of immunoreactivity. Peroxidase activity was visualized with ImmPACT DAB (Brown). Hematoxylin (blue) was used as the nuclear counterstain. Staining was viewed with an E-800 Eclipse microscope (Nikon). TUNEL staining and confocal microscopy Cells were treated as indicated and then fixed in 4% ( w / v ) paraformaldehyde for 15 min. Fixed cells were stained using the DeadEnd Fluorometric TUNEL System (Promega) and Hoechst 33342 (Sigma) according to the manufacturer’s instructions. Confocal images were captured using the × 40 objective on the Olympus Fluoview System laser scanning microscope equipped with the appropriate filter sets and analysed using Photoshop 8.0 and SPOT 3.5 software. Statistical analysis Student’s t -test and two-way ANOVA were used, where appropriate, for statistical analysis. How to cite this article: Yang, S. et al . Pellino3 targets RIP1 and regulates the pro-apoptotic effects of TNF-a. Nat. Commun. 4:2583 doi: 10.1038/ncomms3583 (2013).